The cell cycle regulator GpsB functions as cytosolic adaptor for multiple cell wall enzymes Bacterial growth and cell division requires precise spatiotemporal regulation of the synthesis and remodelling of the peptidoglycan layer that surrounds the cytoplasmic membrane. GpsB is a cytosolic protein that affects cell wall synthesis by binding cytoplasmic mini-domains of peptidoglycan synthases to ensure their correct subcellular localisation. Here, we describe critical structural features for the interaction of GpsB with peptidoglycan synthases from three bacterial species ( Bacillus subtilis , Listeria monocytogenes and Streptococcus pneumoniae ) and suggest their importance for cell wall growth and viability in L. monocytogenes and S. pneumoniae . We use these structural motifs to identify novel partners of GpsB in B. subtilis and extend the members of the GpsB interactome in all three bacterial species. Our results support that GpsB functions as an adaptor protein that mediates the interaction between membrane proteins, scaffolding proteins, signalling proteins and enzymes to generate larger protein complexes at specific sites in a bacterial cell cycle-dependent manner. Peptidoglycan (PG), a network of glycan strands connected by short peptides, forms the essential cell envelope that maintains cell shape and protects bacteria from osmotic stresses [1] . High molecular weight (HMW) bi-functional penicillin binding proteins (class A PBPs) are PG synthases that catalyse glycan strand polymerisation and peptide crosslinking, whereas HMW class B mono-functional PBPs only have transpeptidase functions [2] . The PG layer needs remodelling to enable normal cell growth and division and thus the bacterial cell cycle requires the extracellular activities of PBPs [3] and PG hydrolases [4] to be co-ordinated. The outer membrane-anchored LpoA/B lipoproteins activate their cognate PBP1A/1B PG synthases in the synthesis of the thin, periplasmic PG layer in the Gram-negative paradigm Escherichia coli [5] , [6] . By contrast, Gram-positive bacteria have a much thicker PG layer that is complemented with other anionic cell wall polymers. PG synthesis regulation in Gram-positive bacteria involves protein phosphorylation by orthologues of the serine/threonine kinase PknB [7] /StkP [8] , and dedicated cell cycle scaffolding proteins including DivIVA [9] , EzrA [10] and GpsB [11] , [12] . However, the molecular mechanisms that modulate PG synthesis in Gram-positive bacteria are virtually unknown. GpsB has emerged as a major regulator of PG biosynthesis in low G+C Gram-positive bacteria, and its homologues (DivIVA/Wag31/antigen 84) in Actinobacteria play essential roles in hyphal growth and branching [13] , [14] , [15] . GpsB was initially characterised in Bacillus subtilis where severe cell division and growth defects were observed when both gpsB and ezrA [11] or gpsB and ftsA [12] were deleted. Both EzrA and FtsA play roles in the dynamics and membrane anchoring of the FtsZ Z-ring, the constriction of which is fundamental to cell division [16] . The Z-ring also recruits downstream proteins, including PBPs [17] , [18] , to complete the process. Deletion of gpsB alone in Listeria monocytogenes caused marked growth and division defects at 37 °C and was lethal at 42 °C [19] . Moreover, gpsB deletion in L. monocytogenes also resulted in enhanced susceptibility to β-lactam [19] and fosfomycin [20] antibiotics, reduced virulence in an insect infection model [19] , and caused alterations to PG structure [21] . Mutations in gpsB that affected binding to the PG synthase PBPA1 also showed a lethal phenotype in L. monocytogenes at 42 °C [19] . The gpsB gene is essential in the Streptococcus pneumoniae D39 progenitor strain as well as in some of its laboratory derivatives and its inactivation resulted in elongated cells unable to divide [22] , [23] , [24] . In addition, a genome-wide association study of S. pneumoniae clinical isolates revealed that the presence of gpsB variants was correlated significantly to β-lactam resistance [25] , suggesting that GpsB may have fitness and pleiotropic roles in maintaining cell wall integrity during antibiotic stress. The gpsB gene has also been described as essential in the spherical bacterium Staphylococcus aureus , but the biochemical properties and physiological functions of S. aureus GpsB in this recent report [26] differ to what has been described in B. subtilis [11] , [12] , [18] , [19] , [27] L. monocytogenes [19] , [27] and S. pneumoniae [22] , [23] , [24] . In both B. subtilis [11] and L. monocytogenes [19] , the cytosolic GpsB localises to the lateral side walls of newborn, growing cells and to the septum of dividing cells, the same localisation pattern as that of B. subtilis PBP1 [11] . In S. pneumoniae , GpsB localises to mid-cell [22] , the only region of active PG synthesis for both peripheral (side-wall) elongation and cell division in this bacterium. The localisation of GpsB at regions of active PG synthesis allows for the interaction of GpsB with the poorly characterised cytoplasmic mini-domains of PG synthases [11] , [19] , [27] , [28] . S. pneumoniae GpsB ( Sp GpsB) has been found to co-immunoprecipitate with Sp PBP2a, Sp PBP2b and Sp MreC [24] , suggesting these proteins form a complex that is regulated by Sp GpsB [24] . To gain molecular understanding of GpsB function, we report three crystal structures of PBP cytoplasmic mini-domains in complex with GpsB, the first structures of a PG synthase in complex with a cytoplasmic cell cycle regulator. Despite a marked absence of sequence and structural homology, we find that the PBP domains interact with equivalent surfaces in GpsB using an arginine that is conserved in the respective orthologues of the PBPs. The visualisation of each complex permits a comprehensive mutagenesis strategy and functional study to rationalise the role of each interfacial amino acid in the PBP:GpsB pairs. We uncover a sequence motif used by the B. subtilis PG synthase to interact with GpsB. We identify two new members of the GpsB interactome in this organism by querying the B. subtilis proteome with this motif for potential new partners of GpsB, and provide evidence for their connection to other, established proteins in growth and division. We also identify extensive GpsB interactomes in B. subtilis , L. monocytogenes and S. pneumoniae by bacterial two-hybrid assays (BACTH). Therefore, the role of GpsB in the bacterial cell cycle is that of an adaptor [29] , [30] , [31] , docking PG synthases to other cell wall enzymes, scaffolds and shape determinants into protein complexes for division (the divisome) and peripheral growth (the elongasome). The first 16 residues of Bs PBP1 dictate the Bs GpsB interaction GpsB is an influential cell cycle regulator in low G+C Gram-positive bacteria and we set out to establish the common rules by which GpsB interacts with major PG synthases in three important bacteria—one model species ( B. subtilis ) and two pathogens ( L. monocytogenes and S. pneumoniae ). It has been determined previously by us by SPR that the first 31 amino acids of the cytoplasmic mini-domain of B. subtilis PBP1 ( Bs PBP1) were critical for binding of Bs GpsB [19] . Using the same technique the binding site was further mapped to the first 16 amino acids of Bs PBP1 by comparing the interaction of Bs GpsB with SPR chips coated with full-length Bs PBP1 and a PBP1 deletion mutant, Bs PBP1 17-914 , where the codons for the first 16 amino acids were removed genetically. While submicromolar concentrations of Bs GpsB bound to chips coated with the wild-type Bs PBP1, there was no interaction even when 25 µM Bs GpsB was injected over equivalent chips coated with Bs PBP1 17-914 (Fig. 1a ). Fig. 1 Bs GpsB: Bs PBP1 interactions require conserved arginines in the α-helical cytoplasmic minidomain of Bs PBP1. a Bs GpsB interacts with the first 16 amino acids of Bs PBP1. SPR sensorgrams of full-length Bs GpsB against immobilised full-length Bs PBP1 (black) and Bs PBP1 17-914 (red). Bs GpsB does not interact with the Bs PBP1 17-914 coated chip, even when 25 μM GpsB is injected. b Cartoon (left) and surface representation (right) of the crystal structure of the Bs GpsB 5-64 : Bs PBP1 1-17 complex. Bs GpsB 5-64 is coloured cyan and Bs PBP1 1-17 is coloured green and the likely plane of the bacterial membrane is shown as a red box. c The Bs GpsB 5-64 : Bs PBP1 1-17 complex is dependent upon a conserved SRxxR(R/K) motif in Bs PBP1. Key interfacial residues in the Bs GpsB 5-64 : Bs PBP1 1-17 complex are shown as sticks and coloured (and labelled) blue and green, respectively. The carbonyl oxygens of Bs GpsB Ile13 , Bs GpsB Leu14 and Bs GpsB Lys16 are labelled with their respective red numerals. Hydrogen bonds are shown as black dashed lines and the van der Waals’ interactions between Bs GpsB Leu34 and Bs PBP1 Arg8 are in yellow. d Mutation of key Bs PBP1 interfacial residues in the structure of Bs GpsB 5-64 : Bs PBP1 1-17 leads to a loss of binding of position 16 TAMRA-labelled Bs PBP1 1-32 variants to Bs GpsB 1-68 as measured by fluorescence polarisation. When the Bs PBP1 1-32 peptide was labelled with fluorescein at position 31 the measured affinity was the same as if the fluorophore was at position 16, indicating that the fluorophore itself or its position in the peptide has no impact on the binding interaction. 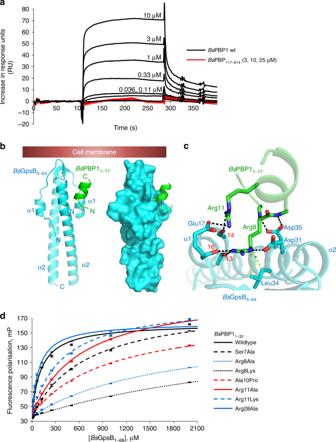Fig. 1 BsGpsB:BsPBP1 interactions require conserved arginines in the α-helical cytoplasmic minidomain ofBsPBP1.aBsGpsB interacts with the first 16 amino acids ofBsPBP1. SPR sensorgrams of full-lengthBsGpsB against immobilised full-lengthBsPBP1 (black) andBsPBP117-914(red).BsGpsB does not interact with theBsPBP117-914coated chip, even when 25 μM GpsB is injected.bCartoon (left) and surface representation (right) of the crystal structure of theBsGpsB5-64:BsPBP11-17complex.BsGpsB5-64is coloured cyan andBsPBP11-17is coloured green and the likely plane of the bacterial membrane is shown as a red box.cTheBsGpsB5-64:BsPBP11-17complex is dependent upon a conserved SRxxR(R/K) motif inBsPBP1. Key interfacial residues in theBsGpsB5-64:BsPBP11-17complex are shown as sticks and coloured (and labelled) blue and green, respectively. The carbonyl oxygens ofBsGpsBIle13,BsGpsBLeu14andBsGpsBLys16are labelled with their respective red numerals. Hydrogen bonds are shown as black dashed lines and the van der Waals’ interactions betweenBsGpsBLeu34andBsPBP1Arg8are in yellow.dMutation of keyBsPBP1 interfacial residues in the structure ofBsGpsB5-64:BsPBP11-17leads to a loss of binding of position 16 TAMRA-labelledBsPBP11-32variants toBsGpsB1-68as measured by fluorescence polarisation. When theBsPBP11-32peptide was labelled with fluorescein at position 31 the measured affinity was the same as if the fluorophore was at position 16, indicating that the fluorophore itself or its position in the peptide has no impact on the binding interaction. The calculated dissociation constants can be found in Supplementary Table1 The calculated dissociation constants can be found in Supplementary Table 1 Full size image We subsequently solved the crystal structure of the complex between the N-terminal domain of Bs GpsB whose termini were truncated slightly to expedite crystallisation, Bs GpsB 5-64 , with the first 17 amino acids of Bs PBP1, Bs PBP1 1-17 (Fig. 1b, c ). The Bs PBP1 1-17 α-helix is stabilised by an intramolecular salt bridge between Bs PBP1 1-17 Glu9 and Bs PBP1 1-17 Arg12 and by a hydrogen bond between the sidechain of Bs PBP1 1-17 Ser7 and the backbone amide of Bs PBP1 1-17 Ala10 . A prominent feature of the complex is the deep penetration of the sidechain of Bs PBP1 Arg8 into the groove between Bs GpsB 5-64 α-helices 1 and 2, contacting the mainchain carbonyl oxygens of Bs GpsB Ile13 , Bs GpsB Leu14 and Bs GpsB Lys16 and forming a salt bridge with Bs GpsB Asp31 (Fig. 1c ), which in turn is tethered in place by hydrogen bonds to the hydroxyl of Bs GpsB Tyr25 . The backbone amides of Bs PBP1 Arg8 and Bs PBP1 Glu9 interact with Bs GpsB Asp35 , mimicking the mainchain interactions in successive turns in an α-helix. In a longer α-helix, the backbone amides of Bs PBP1 Arg8 and Bs PBP1 Glu9 would not be available to interact with Bs GpsB Asp35 because of intra-helical hydrogen bonds with the mainchain carbonyls of Bs PBP1 Phe5 and Bs PBP1 Asn6 . The sidechain of Bs PBP1 Arg11 forms hydrogen bonds with the carbonyl oxygen of Bs GpsB Leu14 and a salt bridge with Bs GpsB Glu17 . Van der Waals’ interactions connect Bs PBP1 Arg8 to Bs GpsB Leu34 (Fig. 1c ) and Bs PBP1 Glu9 with Bs GpsB Lys32 . The Bs PBP1 1-17 peptide binds to a groove between α-helices 1 and 2 in only one molecule of Bs GpsB 5-64 in the crystallographic asymmetric unit as the second Bs GpsB-binding site is blocked by crystal contacts. The key interactions are mapped onto GpsB and PBP1 sequences in Supplementary Figure 1A . To rationalise the features of PBP cytoplasmic domains important for determining recognition by GpsB, the interactions described above were analysed further by fluorescence polarisation (FP) and circular dichroism (CD). The Bs GpsB 1-68 Glu17Ala , Bs GpsB Tyr25Phe , Bs GpsB 1-68 Asp31Ala and Bs GpsB 1-68 Asp35Ala mutations had little impact on protein stability (Supplementary Figure 1B and Supplementary Note 1 ) and each reduced the affinity for Bs PBP1 1-32 by more than 8-fold (Supplementary Figure 1C , Supplementary Table 1 ). Bs PBP1 Arg8Lys , Bs PBP1 Arg8Ala and Bs PBP1 Arg11Ala mutations each resulted in reduced affinities for Bs GpsB 1-68 by at least 5-fold (Fig. 1d , Supplementary Table 1 ). Bs PBP1 1-32 Arg28Ala had no effect on binding (Fig. 1d , Supplementary Table 1 ), suggesting that the overall positive charge of the peptide is not the primary determinant of Bs GpsB: Bs PBP1 interactions, rather the unique physicochemical characteristics of an arginine at position 8 in Bs PBP1 is essential. The Bs PBP1 1-32 Ser7Ala and Bs PBP1 1-32 Ala10Pro mutations each reduced the affinity for Bs GpsB 1-68 by at least 6-fold by affecting the α-helix of BsPBP11-32 (Fig. 1d , Supplementary Figure 1D , Supplementary Table 1 and Supplementary Note 1 ), and the reduction in affinity was the same irrespective of the position of the fluorophore in the peptide (Supplementary Figure 1E , Supplementary Table 1 ). Bs PBP1 1-32 Ser7 acts as the helix N-cap, a role that is performed preferentially by Ser, Asn and Thr [32] , and alanine and proline substitutions in helical positions equivalent to Bs PBP1 1-32 Ser7 and Bs PBP1 1-32 Ala10 , respectively, destabilise model peptides [32] , [33] . Finally, the importance of Bs PBP1 1-32 Ser7 , Bs PBP1 1-32 Arg8 and Bs PBP1 1-32 Arg11 to GpsB binding is highlighted because these are the most well conserved residues in an alignment of the cytoplasmic mini-domains of Bacillaceae PBP1 PG synthases (Supplementary Figure 1F ). L. monocytogenes GpsB interacts with PBPA1 by a TRxxYR motif The deletion of gpsB alone in B. subtilis has no readily apparent phenotype until combined with deletions in ezrA [11] or ftsA [12] ; by contrast, the deletion of gpsB in L. monocytogenes is lethal when grown at 42 °C [19] . Since GpsB in both species interact with class A PG synthases, we next determined whether the rules established above for the Bs GpsB: Bs PBP1 interaction could be applied directly to Lm GpsB: Lm PBPA1. The cytoplasmic mini-domain of Lm PBPA1, Lm PBPA1 1-29 , has an abundance of positively charged residues, but lacks an exact copy of the SRxxR(R/K) motif of Bacillaceae PBP1 (Supplementary Figure 1 F, 2A ); the closest equivalent is TRxxYR. 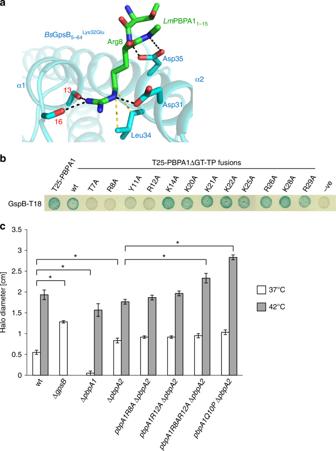Fig. 2 TheLmGpsB:LmPBPA1 interactions are also governed by a conserved arginine.aThe structure of theBsGpsB5-64Lys32Glu:LmPBPA11-15complex reveals that only Arg8 and adjacent backbone atoms of theLmPBPA11-15peptide are ordered. In this cartoon,BsGpsB5-64Lys32Gluis coloured cyan and selected sidechains are drawn as stick with cyan carbons, whereas theLmPBPA11-15peptide is represented in stick form, with green carbons. The carbonyl oxygens ofBsGpsBIle13andBsGpsBLys16are denoted by respective red numerals. Hydrogen bonds are shown as black dashed lines and the van der Waals’ interactions betweenBsGpsBLeu34andLmPBPA1Arg8are in yellow. Only one PBP-binding site is occupied by peptide in these crystals because the second site is blocked by crystal contacts.bMutation of conservedLmPBPA1 residues results in a loss of interaction by BACTH. The removal of residues 92–827, correlating to the glycosyltransferase and transpeptidase domains ofLmPBPA1, results in the PBPA1ΔGT-TP peptide. Empty pKT25 (−) was used as a negative control. Agar plates were photographed after 24 h at 30 °C.cEffect of N-terminalpbpA1mutations on fosfomycin sensitivity of a ΔpbpA2mutant. Wild-type and mutantL. monocytogenesEGD-e strains were grown as confluent layers on BHI agar plates at 37 °C and 42 °C and halo diameters around fosfomycin-containing filter discs were measured and corrected for the disc diameter. The experiment was performed in triplicate, and average values and standard deviations are shown. Asterisks indicate statistically significant differences (P< 0.01,t-test) In FP, the first 20 amino acids of Lm PBPA1, Lm PBPA1 1-20 , bound to the N-terminal domain of Lm GpsB, Lm GpsB 1-73 , with an affinity similar to that of Bs PBPA1 1-32 for Bs GpsB 1-68 (Supplementary Figure 2B , Supplementary Table 1 ), but we were unable to co-crystallise Lm GpsB constructs with Lm PBPA1 peptides to visualise these interactions and to compare them to Bs GpsB 5-64 : Bs PBP1 1-17 . Consequently, and to expedite crystallisation, we solved the structure of the first 15 amino acids of Lm PBPA1, Lm PBPA1 1-15 , bound to Bs GpsB 5-64 Lys32Glu , which is a surrogate for Lm GpsB 1-73 because (i) all the residues within 8 Å of the Bs GpsB 5-64 : Bs PBP1 1-17 interface are conserved in Lm GpsB except for Lys32, which is glutamate in Lm GpsB, and thus all peptide-contacting residues are maintained—as well as bystander residues that help indirectly to shape the PBP binding site; (ii) Lm GpsB and Bs GpsB use overlapping PBP binding sites [19] ; (iii) the K d s of Bs GpsB 1-68 Lys32Glu and Lm GpsB 1-73 for the first 20 amino acids of Lm PBPA1, Lm PBPA1 1-20 , are almost identical (Supplementary Figure 2B , Supplementary Table 1 ). Therefore, the K32E variant of the N-terminal domain of Bs GpsB is as close a surrogate for the equivalent Lm GpsB domain that could be obtained. The subsequent structure of the Bs GpsB 5-64 Lys32Glu : Lm PBPA1 1-15 complex revealed that, in contrast to the Bs GpsB 5-64 : Bs PBP1 1-17 complex, the majority of the Lm PBPA1 peptide was disordered except for Lm PBPA1 1-15 Arg8 and the immediately-adjacent mainchain atoms. Lm PBPA1 1-15 Arg8 adopts the same orientation and makes the same interactions as described above for Bs PBP1 1-17 Arg8 in the Bs GpsB 5-64 : Bs PBP1 1-17 complex (Figs. 1 c, 2a ). The bidentate interaction of Glu35 of Bs GpsB 5-64 Lys32Glu with the backbone amides of Lm PBPA1 Arg8 and Lm PBPA1 Ser9 are maintained just as in the Bs GpsB 5-64 : Bs PBP1 1-17 complex and, as the backbone torsion angles of Lm PBPA1 1-15 Arg8 are also α-helical, it suggests that the role of the conserved Lm PBPA1 Thr7 is to N-cap this helix [32] . The interaction of Bs GpsB 5-64 Lys32Glu with Lm PBPA1 1-15 seemingly centres almost entirely on a single arginine. How Lm GpsB discerns Lm PBPA1 Arg8 over other positively charged residues in the arginine- and lysine-rich cytoplasmic domain of Lm PBPA1 (Supplementary Figure 2A ) was determined by FP and BACTH. Lm PBPA1 1-20 Arg8Ala and Lm PBPA1 1-20 Arg12Ala mutations reduced the affinity for Bs GpsB 1-68 Lys32Glu by >15- and ~4-fold, respectively (Supplementary Figure 2B , Supplementary Table 1 ), and had significant negative impact on the Lm GpsB: Lm PBPA1 interaction by BACTH (Fig. 2b ). Alanine substitution of Lm PBPA1 Tyr11 had a comparatively milder impact in BACTH (Fig. 2b ) and in FP (Supplementary Figure 2B , Supplementary Table 1 ). Reintroducing positive charge into Lm PBPA1 1-20 Arg8Ala did not restore wild-type binding affinity in FP as Lm PBPA1 1-20 Arg8Ala,Ser16Arg still bound to Bs GpsB 1-68 Lys32Glu with an affinity at least 10-fold weaker than wild-type (Supplementary Figure 2B , Supplementary Table 1 ). BACTH also supports the central importance of Lm PBPA1 Thr7 , which presumably plays a structural role in the Lm PBPA1 1-15 peptide possibly by acting as an N-cap and positioning Lm PBPA1 Arg8 at the start of an α-helix at the. Alanine substitution of the other positively charged residues downstream of residue 14 had no impact in BACTH (Fig. 2b ), consistent with the particularly stringent specificity of Lm GpsB for Lm PBPA1 Arg8 in comparison to other positively charged residues. Fig. 2 The Lm GpsB: Lm PBPA1 interactions are also governed by a conserved arginine. a The structure of the Bs GpsB 5-64 Lys32Glu : Lm PBPA1 1-15 complex reveals that only Arg8 and adjacent backbone atoms of the Lm PBPA1 1-15 peptide are ordered. In this cartoon, Bs GpsB 5-64 Lys32Glu is coloured cyan and selected sidechains are drawn as stick with cyan carbons, whereas the Lm PBPA1 1-15 peptide is represented in stick form, with green carbons. The carbonyl oxygens of Bs GpsB Ile13 and Bs GpsB Lys16 are denoted by respective red numerals. Hydrogen bonds are shown as black dashed lines and the van der Waals’ interactions between Bs GpsB Leu34 and Lm PBPA1 Arg8 are in yellow. Only one PBP-binding site is occupied by peptide in these crystals because the second site is blocked by crystal contacts. b Mutation of conserved Lm PBPA1 residues results in a loss of interaction by BACTH. The removal of residues 92–827, correlating to the glycosyltransferase and transpeptidase domains of Lm PBPA1, results in the PBPA1ΔGT-TP peptide. Empty pKT25 (−) was used as a negative control. Agar plates were photographed after 24 h at 30 °C. c Effect of N-terminal pbpA1 mutations on fosfomycin sensitivity of a Δ pbpA2 mutant. Wild-type and mutant L. monocytogenes EGD-e strains were grown as confluent layers on BHI agar plates at 37 °C and 42 °C and halo diameters around fosfomycin-containing filter discs were measured and corrected for the disc diameter. The experiment was performed in triplicate, and average values and standard deviations are shown. Asterisks indicate statistically significant differences ( P < 0.01, t -test) Full size image Lm PBPA1 Arg8 and Bs PBP1 Arg8 are equivalent in their interactions with GpsB. Of the other GpsB-binding determinants of Bs PBP1, Lm PBPA1 lacks an analogous Bs PBP1 Arg11 . The sequential equivalent is Lm PBPA1 Tyr11 , but this residue is completely disordered and its mutation to alanine reduced the affinity for Bs GpsB 1-68 Lys32Glu only by 2-fold (Supplementary Figure 2B ). To further decipher the reason for the specificity for Lm PBPA1 Arg8 , the importance of α-helix formation in Lm PBPA1 1-15 for GpsB binding was analysed with Q10P-mutated Lm PBPA1 peptides. A Q10P mutation caused a >7-fold reduction in binding affinity (Supplementary Figure 2B , Supplementary Table 1 ) and CD confirmed a significant impact of the Q10P mutation on the α-helicity of Lm PBPA1 1-15 peptides (Supplementary Figure 2C ). Finally, the effects of mutations to the crucial Lm GpsB-interacting residues in Lm PBPA1 were also probed in Listeria using fosfomycin sensitivity as a reporter since Δ gpsB mutants are more susceptible to this antibiotic at 37 °C than wild-type L. monocytogenes [20] . Fosfomycin inhibits the first enzyme in the biosynthetic pathway of PG, MurA, and the Δ gpsB mutant is hypersensitive to it probably because of unproductive consumption of PG precursors due to mis-regulated Lm PBPA1 [20] . By contrast, removal of pbpA1 reduces substrate turnover in PG biosynthesis and thus the cells become more resistant to fosfomycin, and a pbpA1 pbpA2 double mutant is not viable [34] . Effects on fosfomycin sensitivity were apparent in mutants carrying the pbpA1 Arg8Ala,Arg12Ala and pbpA1 Gln10Pro alleles but only when Lm PBPA2, the Lm PBPA1 paralogue, was also absent (Fig. 2c ). Synthetic lethality with pbpA2 and a growth defect at 42 °C is characteristic of the L. monocytogenes null gpsB mutant [19] , suggesting that the observed effects partially phenocopy Δ gpsB . However, no pbpA1 mutation phenocopied the Δ gpsB mutant completely (Supplementary Figure 2D ). Taken together, our data highlight the importance of a conserved arginine and α-helicity in class A PG synthases for interacting with GpsB in two species. In both cases the arginine is adjacent to a conserved residue with high propensity to act as a helix N-cap, implying that positioning of the arginine at the start of the helix is critical. Furthermore, since pbpA1 does not phenocopy gpsB in L. monocytogenes , and gpsB deletion on its own in B. subtilis has no clear phenotype, GpsB must have additional functions in both bacteria. Extending the B. subtilis and L. monocytogenes GpsB interactomes The data presented above describe features critical for interactions involving Bs GpsB, which include a helical SRxxR(R/K) motif in close proximity to the membrane. To identify hitherto unidentified Bs GpsB-interacting proteins, the B. subtilis proteome was queried with the SRxxR(R/K) motif. Two previously uncharacterised ORFs, Bs YpbE and Bs YrrS, conform to all the features described above. Bs YpbE is a membrane protein with a 56-residue cytoplasmic domain that encodes a SRVERR motif. The extracellular region, residues 80–240, contains a LysM (lysin motif) domain between residues 189 and 235; LysM domains are ~40-residue, degenerate PG- and chitin-binding modules widespread in bacteria and eukaryotes. yrrS is found in a bicistronic operon widely conserved in the Bacillaceae with the gene ( yrrR ) encoding a class B PBP, PBP4b [35] , suggesting these genes have a linked function in cell wall homoeostasis [36] . Bs YrrS comprises an 18-residue cytoplasmic domain with two potential, overlapping Bs GpsB-binding motifs SRYENR and NRDKRR and an extracellular domain that belongs to the widespread and currently uncharacterised DUF1510 family. LysM domains are frequently found as tandem repeats within bacterial proteins [37] and the individual domains can act co-operatively to bind PG [38] , [39] . Bs YpbE contains one LysM domain hence oligomerization of Bs YpbE may enhance PG binding, with the oligomerisation of the extracellular LysM domain of Bs YpbE presumably controlled by cytoplasmic, hexameric Bs GpsB [27] , the essential form of the protein in bacteria [19] . In the absence of purified, full-length Bs YpbE to test this hypothesis directly, monomeric and dimeric forms of Bs YpbE 130-240 , which encompasses the sole extracellular LysM domain, were generated instead. Dimeric Bs YpbE 130-240 was prepared by mutation of Ser132 to cysteine to enable disulphide-linked Bs YpbE 130-240 Ser132Cys dimers to be purified. 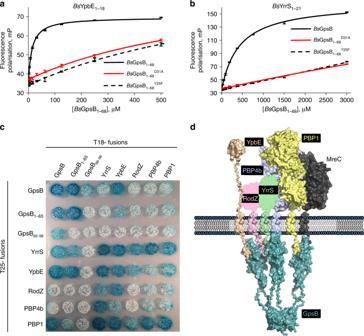Fig. 3 The SRxxR(R/K) motif identifiesBsYpbE andBsYrrS as newBsGpsB binding partners.a,bBsYpbE1-18andBsYrrS1-21bind toBsGpsB1-68at the same site asBsPBP1. Fluorescence polarisation ofBsGpsB1-68binding to fluorescein-labelledBsYpbE1-18(a) and fluorescein-labelledBsYrrS1-21(b). The interaction of wild-type proteins is depicted by black curves, whereas the red curves and dashed black lines correspond toBsGpsB1-68Asp31AlaandBsGpsB1-68Tyr25Phemutants, respectively.cBACTH reveals a newBsGpsB interaction network involving proteins encoding the SRxxR(R/K) motif. The panel shows pairwise combinations of proteins expressed as N-terminal fusions to both halves of adenylate cyclase in the BACTH host strain. Their presence in complexes containingBsRodZ,BsPBP4b andBsPBP1 imply roles forBsYrrS andBsYpbE in sidewall synthesis during cell growth. The validity of the observed interactions is supported by the behaviour of the T18-GpsB66-98fusion, which does not interact with any other partner except T25-GpsB, and therefore acts as an internal control. The T18-BsGpsB66-98:T25-BsGpsB interaction is consistent with the hexameric nature ofBsGpsB19,26. The absence of interactions betweenBsGpsB66-98andBsYrrS orBsYpbE is consistent with data inbthat shows that the N-terminal domain of GpsB interacts with the SRxxR(R/K) motif of YpbE and YrrS.dA model recapitulates interactions betweenBsGpsB and partners. Surface representations of the SAXS structure ofLmGpsB26(coloured teal) and the closest homologues in the PDB by sequence (BsPBP1, yellow, PDBid2OLV;BsPBP4b, pale blue,4L0L;BsRodZ, pink,2WUS;BsMreC, dark grey,2J5U;BsYpbE, salmon,2MKXand the linker represents the disordered region, residues 131-188) are used as models for theB. subtilisproteins. Amorphous blobs, the surface area of which are scaled proportional to molecular weight, are used forBsYrrS (green) and the extracellular domain ofBsRodZ (pink) where there is no structural information. The N-terminal domain of each membrane protein is cytoplasmic and 22-amino acid model helices represent each TM helix. The TMpred-predicted TM boundaries are:BsPBP1 (38-60);BsPBP4b (9-31);BsYrrS (19-41);BsYpbE (57-79);BsRodZ (89-111) andBsMreC (7-24). The GpsB-interacting domains ofBsYpbE,BsYrrS andBsPBP1 are based on theBsPBP11-17structure In pulldown assays, the binding of Bs YpbE 130-240 Ser132Cys dimers to PG was enhanced considerably relative to the monomeric, cysteine-free version of Bs YpbE 130-240 (Supplementary Figure 3A ). Therefore, the binding of YpbE to PG in B. subtilis will be stimulated by YpbE multimerisation, induced by hexameric GpsB. The interaction of Bs GpsB 1-68 with Bs YrrS and Bs YpbE was assessed by FP and BACTH. Bs GpsB 1-68 bound to a 21-residue fragment of the cytoplasmic domain of Bs YpbE, Bs YpbE 1-21 that encompasses the SRVERR motif, and the entire cytoplasmic mini-domain of Bs YrrS, Bs YrrS 1-18 , with K d values of 13 μM (Fig. 3a ) and 430 μM (Fig. 3b ), respectively. The modest affinity of the Bs YrrS 1-18 peptide for Bs GpsB 1-68 (Supplementary Table 1 ) probably translates to a substantially tighter affinity in bacterial cells, because of an avidity effect resulting from Bs GpsB and Bs YrrS associating with membranes, effectively increasing the local concentration of each significantly. The specificity of these interactions measured by FP was consistent with the impact of Bs GpsB Asp31Ala and Bs GpsB Tyr25Phe mutations, each of which reduced the affinities for Bs YrrS 1-18 and Bs YpbE 1-21 by 7- and ~40-fold, respectively (Fig. 3a, b ), and in-line with the roles of Bs GpsB Asp31 and Bs GpsB Tyr25 in defining the Bs PBP1 binding site. Interactions of Bs GpsB with Bs YrrS and Bs YpbE were also detected by BACTH, with the interactions mapping to the N-terminal domain of Bs GpsB in both cases (Fig. 3c ). GpsB is only conditionally essential in B. subtilis [11] , [12] , and perhaps it is not surprising that no obvious cell growth or division phenotypes were identified in our hands or previously [40] on deleting the genes encoding Bs YrrS, Bs PBP4b or Bs YpbE. BACTH was used to confirm that Bs YrrS interacted with Bs PBP4b, Bs PBP1 and Bs RodZ; the latter two proteins have established roles in cell division, growth and morphogenesis [41] , [42] . The interaction between Bs PBP1 and a fragment of Bs YrrS lacking residues 13-16, Bs YrrS Δ13-16 (which reduced non-specific binding to the Bs PBP1-immobilised SPR chip and did not affect the SRYENR motif) was quantified by SPR, and Bs YrrS Δ13-16 bound to Bs PBP1 with a K d of 20 nM (Supplementary Figure 3B ). Therefore, these gene products are capable of forming a network of interactions (Fig. 3d ) that may be nucleated by the formation of a Bs PBP1: Bs YrrS complex. Fig. 3 The SRxxR(R/K) motif identifies Bs YpbE and Bs YrrS as new Bs GpsB binding partners. a , b Bs YpbE 1-18 and Bs YrrS 1-21 bind to Bs GpsB 1-68 at the same site as Bs PBP1. Fluorescence polarisation of Bs GpsB 1-68 binding to fluorescein-labelled Bs YpbE 1-18 ( a ) and fluorescein-labelled Bs YrrS 1-21 ( b ). The interaction of wild-type proteins is depicted by black curves, whereas the red curves and dashed black lines correspond to Bs GpsB 1-68 Asp31Ala and Bs GpsB 1-68 Tyr25Phe mutants, respectively. c BACTH reveals a new Bs GpsB interaction network involving proteins encoding the SRxxR(R/K) motif. The panel shows pairwise combinations of proteins expressed as N-terminal fusions to both halves of adenylate cyclase in the BACTH host strain. Their presence in complexes containing Bs RodZ, Bs PBP4b and Bs PBP1 imply roles for Bs YrrS and B sYpbE in sidewall synthesis during cell growth. The validity of the observed interactions is supported by the behaviour of the T18-GpsB 66-98 fusion, which does not interact with any other partner except T25-GpsB, and therefore acts as an internal control. The T18- Bs GpsB 66-98 :T25- Bs GpsB interaction is consistent with the hexameric nature of Bs GpsB [19] , [26] . The absence of interactions between Bs GpsB 66-98 and Bs YrrS or Bs YpbE is consistent with data in b that shows that the N-terminal domain of GpsB interacts with the SRxxR(R/K) motif of YpbE and YrrS. d A model recapitulates interactions between Bs GpsB and partners. Surface representations of the SAXS structure of Lm GpsB [26] (coloured teal) and the closest homologues in the PDB by sequence ( Bs PBP1, yellow, PDBid 2OLV ; Bs PBP4b, pale blue, 4L0L ; Bs RodZ, pink, 2WUS ; Bs MreC, dark grey, 2J5U ; Bs YpbE, salmon, 2MKX and the linker represents the disordered region, residues 131-188) are used as models for the B. subtilis proteins. Amorphous blobs, the surface area of which are scaled proportional to molecular weight, are used for Bs YrrS (green) and the extracellular domain of Bs RodZ (pink) where there is no structural information. The N-terminal domain of each membrane protein is cytoplasmic and 22-amino acid model helices represent each TM helix. The TMpred-predicted TM boundaries are: Bs PBP1 (38-60); Bs PBP4b (9-31); Bs YrrS (19-41); Bs YpbE (57-79); Bs RodZ (89-111) and Bs MreC (7-24). The GpsB-interacting domains of Bs YpbE, Bs YrrS and Bs PBP1 are based on the Bs PBP1 1-17 structure Full size image Homologues of YpbE do not exist in L. monocytogenes and the YrrS homologue (Lmo1495) does not contain a signature Bs GpsB-binding motif and neither protein is found in S. pneumoniae . No strong potential GpsB-interacting candidates were identified when the L. monocytogenes proteome was searched with either TRxxYR or SRxxR(R/K) as the query. BACTH was thus used to uncover additional potential Lm GpsB functions in L. monocytogenes using a bank of 27 listerial components from the known elongation and division machineries in bacteria (Supplementary Note 2 ). Twelve proteins were shown to interact with Lm GpsB and only these are shown in Supplementary Figure 3C . There is no consensus motif shared by these proteins, though all have at least one arginine present in their cytoplasmic regions that is conserved in their respective orthologues. Two classes of hits were identified in the BACTH screen; class I hits ( Lm PBPA1, Lm MreC and Lm SepF, and Lm GpsB self-interactions) turned blue after one day of incubation (Supplementary Figure 3C ). Class II hits turned blue after 2 days incubation at 30 °C, including Lm ZapA, Lm EzrA, Lm DivIB, Lm DivIC, Lm MreC, Lm MreBH and the other HMW Lm PBPs (Supplementary Figure 3C ). All of these interactions, except for the GpsB self-interactions, required the Lm GpsB N-terminal domain (Supplementary Figure 3C ). In good agreement with the absence of a TRxxYR motif in Lm MreC, Lm SepF and Lm ZapA, interactions with these proteins did not require key residues in the known PBP-binding groove in Lm GpsB (Supplementary Figure 3D ) and reciprocal tests validated the Lm GpsB: Lm PBPA1 interactions [21] . It would thus seem that Lm PBPA1 represents the only GpsB binding partner that employs the TRxxYR motif in L. monocytogenes . Two arginines dictate S. pneumoniae GpsB:PBP2a molecular recognition S. pneumoniae , more distantly related to either Bacillus or Listeria , is an ovoid-shaped Gram-positive coccus in which GpsB is essential [22] , [23] , [24] . Sp GpsB co-immunoprecipitated with Sp PBP2a (one of three pneumococcal class A PBPs), Sp MreC and other proteins, suggesting they interact at some point in the pneumococcal cell cycle [24] . Synthetic lethality studies in pneumococcal Δ gpsB suppressor mutants revealed that pbp1a , and not pbp2a , became essential in the absence of gpsB indicating that Sp PBP2a is the class A PBP regulated by Sp GpsB in S. pneumoniae [24] . 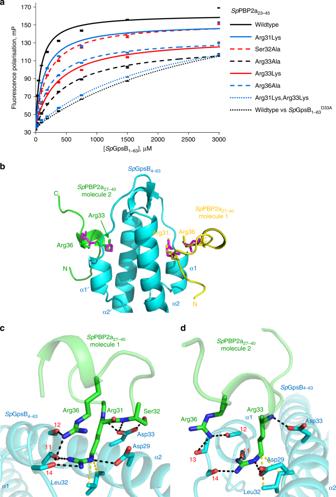Fig. 4 TheSpPBP2a minidomain is not α-helical but still interacts withSpGpsB through conserved arginines.aArginine residues ofSpPBP2a play a key role in binding toSpGpsB. Unless otherwise indicated, the fluorescence polarisation binding curves represent the interaction of TAMRA-labelledSpPBP2a23-45peptides with wildtypeSpGpsB1-63. The relevant dissociation constants are listed in Supplementary Table1.bThe structure of theSpGpsB4-63:SpPBP2a27-40complex reveals the critical role ofSpPBP2a arginines for the interaction withSpGpsB. In this cartoon,SpGpsB4-63is coloured cyan, and theSpPBP2a27-40peptide is coloured yellow (molecule 1) and green (molecule 2). The sidechains of Arg8 and Arg11 from theBsGpsB5-64:BsPBP11-17complex are shown as red sticks after a global superimposition of equivalent GpsB atoms. In molecule 1,SpPBP2aArg31andSpPBP2aArg36superimpose withBsGpsB5-64Arg8andBsGpsB5-64Arg11whereas molecule 2 accommodatesSpPBP2aArg33andSpPBP2aArg36.c,dClose-up view of the interactions ofSpPBP2a from molecule 1 (c) and 2 (d) withSpGpsB4-63. Key interfacial sidechains and backbone atoms are represented in stick format;SpGpsB4-63is coloured cyan andSpPBP2A27-40is coloured green. The van der Waals’ interactions betweenSpGpsBLeu32andSpPBP1Arg31(molecule 1) andSpPBP1Arg33(molecule 2) are in yellow. The carbonyl oxygens ofSpGpsBIle11,SpGpsBPhe12,SpGpsBGlu13andSpGpsBGln14are denoted by respective red numerals We found that the cytoplasmic mini-domain of Sp PBP2a and many of its orthologues contain the consensus sequence (S/R)RS(R/G)(K/S)xR (Supplementary Figure 4A ) that resembles the Bacillaceae PBP1 SRxxR(R/K) motif (Supplementary Figure 1F ). A 22-residue peptide of Sp PBP2a that encompasses this region, Sp PBP2a 23-45 , was found by FP to bind to the N-terminal domain of Sp GpsB, Sp GpsB 1-63 , with a K d of 80 μM whereas Sp GpsB 1-63 Asp33Ala (equivalent to Bs GpsB Asp35Ala ) had a ~40-fold reduced affinity for Sp PBP2a 23-45 (Fig. 4a , Supplementary Table 1 ). The crystal structure of a slightly truncated form of the N-terminal domain of Sp GpsB, Sp GpsB 4-63 (to expedite crystallisation), was solved in the presence of a 14-residue peptide of Sp PBP2a, Sp PBP2a 27-40 , which includes the (S/R)RS(R/G)(K/S)xR motif. In this instance, each subunit of the Sp GpsB dimer is peptide-bound (Fig. 4b ). Peptide binding principally involves two arginines but each Sp GpsB subunit recognises the peptide differently. In Sp GpsB 4-63 molecule 1, Sp PBP2a 27-40 recognition centres on Sp PBP2a Arg31 and Sp PBP2a Arg36 (Fig. 4c ), whereas molecule 2 involves Sp PBP2a Arg33 and Sp PBP2a Arg36 (Fig. 4d ). The arginine pairs occupy the same positions as Bs PBP1 Arg11 and Bs PBP1 Arg8 in the Bs GpsB 5-64 : Bs PBP1 1-17 complex (Fig. 1c ); Sp PBP2a Arg36 is equivalent to Bs PBP1 Arg11 whereas Sp PBP2a Arg31 and Sp PBP2a Arg33 are equivalent to Bs PBP1 Arg8 . Fig. 4 The Sp PBP2a minidomain is not α-helical but still interacts with Sp GpsB through conserved arginines. a Arginine residues of Sp PBP2a play a key role in binding to Sp GpsB. Unless otherwise indicated, the fluorescence polarisation binding curves represent the interaction of TAMRA-labelled Sp PBP2a 23-45 peptides with wildtype Sp GpsB 1-63 . The relevant dissociation constants are listed in Supplementary Table 1 . b The structure of the Sp GpsB 4-63 : Sp PBP2a 27-40 complex reveals the critical role of Sp PBP2a arginines for the interaction with Sp GpsB. In this cartoon, Sp GpsB 4-63 is coloured cyan, and the Sp PBP2a 27-40 peptide is coloured yellow (molecule 1) and green (molecule 2). The sidechains of Arg8 and Arg11 from the Bs GpsB 5-64 : Bs PBP1 1-17 complex are shown as red sticks after a global superimposition of equivalent GpsB atoms. In molecule 1, Sp PBP2a Arg31 and Sp PBP2a Arg36 superimpose with Bs GpsB 5-64 Arg8 and Bs GpsB 5-64 Arg11 whereas molecule 2 accommodates Sp PBP2a Arg33 and Sp PBP2a Arg36 . c , d Close-up view of the interactions of Sp PBP2a from molecule 1 ( c ) and 2 ( d ) with Sp GpsB 4-63 . Key interfacial sidechains and backbone atoms are represented in stick format; Sp GpsB 4-63 is coloured cyan and Sp PBP2A 27-40 is coloured green. The van der Waals’ interactions between Sp GpsB Leu32 and Sp PBP1 Arg31 (molecule 1) and Sp PBP1 Arg33 (molecule 2) are in yellow. The carbonyl oxygens of Sp GpsB Ile11 , Sp GpsB Phe12 , Sp GpsB Glu13 and Sp GpsB Gln14 are denoted by respective red numerals Full size image The Sp GpsB: Sp PBP2a interaction was confirmed by BACTH (Supplementary Figure 4B ). The interaction was lost completely with Sp GpsB Tyr23Ala , Sp GpsB Val28Ala , Sp GpsB Asp29Ala , Sp GpsB Leu32Ala and Sp GpsB Asp33Ala mutated proteins and reduced with Sp GpsB Ile36Ala (Fig. 5a ). All the Sp GpsB variants retained the ability to self-interact and to interact with wild-type Sp GpsB (Fig. 5a , Supplementary Figure 4C ); the impact of the mutations on interactions with Sp PBP2a thus does not reflect impaired expression of the relevant fusion proteins. Moreover, all the Sp GpsB variants, except Sp GpsB Asp29Ala , retained some ability to interact with Sp MreC, which was also confirmed to interact with Sp GpsB by BACTH (Fig. 5a , Supplementary Figure 4B ). Fig. 5 Depletion of Sp PBP2a does not phenocopy depletion of Sp GpsB. a Mutations in Sp GpsB differentially affect interactions with Sp PBP2a and Sp MreC. BACTH analysis of the interactions of Sp GpsB-T18 variants with wild-type Sp GpsB, Sp PBP2a and Sp MreC. pKT25/pUT18C and pKT25-zip/pUT18C-zip plasmid pairs were used as negative (−ve) and positive (+ve) controls, respectively. The agar plates were photographed after 40h incubation at 30 °C. b , c Sp GpsB variants that have lost Sp PBP2a binding have a gpsB null growth and morphology phenotype. Representative growth curve of S. pneumoniae strains with ectopic expression of gpsB + under a Zn 2+ -dependent promoter. GpsB variants of Y23A, V28A, L32A and D33A showed a gpsB null growth phenotype ( b ) and elongated cell morphology ( c ) on gpsB depletion. The D29A variant showed an intermediate growth phenotype, which was also obtained with an independent isogenic isolate and with a gpsB D29A -FLAG labelled strain. The I36A strain has a reduced elongation phenotype. All phase‐contrast micrographs are at the same magnification (scale bar = 1 µm). d , e Sp PBP2a depletion does not phenocopy Sp GpsB. Representative growth curves ( d ) and phase-contrast micrographs ( e ) of parent IU1824 (WT, D39 ∆ cps rpsL1 ), IU13444 (∆ pbp1a ), IU14381 ( ∆pbp2a// Δ bgaA ::P Zn - pbp2a + ∆ pbp1a ) and IU14383 ( ∆gpsB// Δ bgaA ::P Zn - gpsB + ∆ pbp1a ). Similar to the depletion of Sp GpsB in S. pneumoniae pbp1a + strains (see panel b ), depletion of Sp GpsB in IU14383 leads to extremely elongated cells, a growth cessation and lysis phenotype. By contrast, depletion of Sp PBP2a in the ∆ pbp1a background (right hand panels) leads to small but mostly ovococcal cells that do not lyse during the time course examined. All phase-contrast micrographs were taken at OD 620 ≈ 0.15 or at the time point marked by arrows in a for IU14381 and IU14383 under zinc depletion and are at the same magnification (scale bar = 1 µm) Full size image Despite differences in the secondary structures of the two independent Sp PBP2a peptides bound to the Sp GpsB 4-63 dimer (Fig. 4b ), the two arginines form a similar network of interactions with Sp GpsB as described for Bs GpsB and Lm GpsB (Figs. 1 c, 2a ) with additional sidechain contacts in molecule 1 between Sp PBP2a Ser32 and Sp GpsB Asp33 (Fig. 4c ), and Sp PBP2a Arg31 and Sp GpsB Tyr23 . The importance of Sp PBP2a Arg31 and Sp PBP2a Arg33 is further supported by their sequence conservation (Supplementary Figure 4A ) and FP (Fig. 4a , Supplementary Table 1 ). Although Sp PBP2a Arg31Lys had only a 2-fold reduced affinity, which probably reflects the ability of Sp PBP2a Arg33 to compensate for the loss of Sp PBP2a Arg31 , the binding affinity of Sp PBP2a Arg31Lys,Arg33Lys was reduced >25-fold relative to wild type. The importance of the Sp GpsB residues involved in the interactions with Sp PBP2a is also consistent with the phenotype because of the severe growth (Fig. 5b ) and morphological defects (Fig. 5c ) of S. pneumoniae strains harbouring the Sp GpsB Tyr23Ala , Sp GpsB Val28Ala , Sp GpsB Asp29Ala , Sp GpsB Leu32Ala and Sp GpsB Asp33Ala alleles even though the mutated proteins were still capable of self-interactions (Supplementary Figure 4C ) and were expressed at wild-type levels (Supplementary Figure 4D ). However, no obvious phenotype was observed in S. pneumoniae strains carrying the corresponding Sp PBP2a Arg31Ala , Sp PBP2a Arg33Ala or Sp PBP2a Arg31Ala,Ser32Ala,Arg36Ala alleles, even when pbp1a was deleted to decouple the effects of mutations in Sp PBP2a from Sp PBP1a activity (Supplementary Table 2 ). 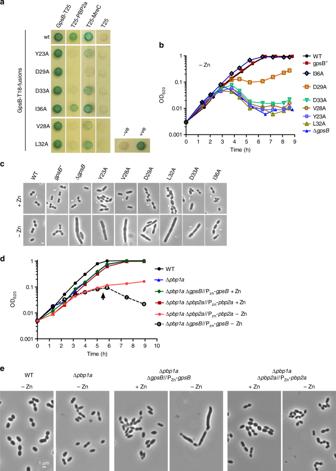Fig. 5 Depletion ofSpPBP2a does not phenocopy depletion ofSpGpsB.aMutations inSpGpsB differentially affect interactions withSpPBP2a andSpMreC. BACTH analysis of the interactions ofSpGpsB-T18 variants with wild-typeSpGpsB,SpPBP2a andSpMreC. pKT25/pUT18C and pKT25-zip/pUT18C-zip plasmid pairs were used as negative (−ve) and positive (+ve) controls, respectively. The agar plates were photographed after 40h incubation at 30 °C.b,cSpGpsB variants that have lostSpPBP2a binding have agpsBnull growth and morphology phenotype. Representative growth curve ofS. pneumoniaestrains with ectopic expression ofgpsB+under a Zn2+-dependent promoter. GpsB variants of Y23A, V28A, L32A and D33A showed agpsBnull growth phenotype (b) and elongated cell morphology (c) ongpsBdepletion. The D29A variant showed an intermediate growth phenotype, which was also obtained with an independent isogenic isolate and with agpsBD29A-FLAG labelled strain. The I36A strain has a reduced elongation phenotype. All phase‐contrast micrographs are at the same magnification (scale bar = 1 µm).d,eSpPBP2a depletion does not phenocopySpGpsB. Representative growth curves (d) and phase-contrast micrographs (e) of parent IU1824 (WT, D39 ∆cps rpsL1), IU13444 (∆pbp1a), IU14381 (∆pbp2a//ΔbgaA::PZn-pbp2a+∆pbp1a) and IU14383 (∆gpsB//ΔbgaA::PZn-gpsB+∆pbp1a). Similar to the depletion ofSpGpsB inS. pneumoniae pbp1a+strains (see panelb), depletion ofSpGpsB in IU14383 leads to extremely elongated cells, a growth cessation and lysis phenotype. By contrast, depletion ofSpPBP2a in the ∆pbp1abackground (right hand panels) leads to small but mostly ovococcal cells that do not lyse during the time course examined. All phase-contrast micrographs were taken at OD620≈ 0.15 or at the time point marked by arrows inafor IU14381 and IU14383 under zinc depletion and are at the same magnification (scale bar = 1 µm) Nevertheless, Sp PBP2a mutants in which amino acids 32–37 or 27–38 or 26–45 were deleted in a Δ pbp1a background showed progressively reduced growth rates in the three deletion strains and pronounced morphological defects in the two strains with larger deletions (Supplementary Figure 5 A, 5B ), despite wild-type levels of protein expression at the respective expected molecular masses (Supplementary Figure 5C ). At least eight residues, including two arginines and one lysine, were retained in all the deletion constructs before the predicted start of the Sp PBP2a TM helix (residue 54), providing the necessary charge to satisfy the inside-positive rule [43] . Consistent with the pbp2a deletion mutant phenotypes, BACTH results for the correspondent truncated Sp PBP2a variants showed reduced interactions with Sp GpsB in comparison to the wildtype but not with Sp MreC (Supplementary Figure 5 D, 5E ). Together, these results support a critical role of the (S/R)RS(R/G)(K/S)xR motif between Sp PBP2a residues 30 and 36 for mediating protein–protein interactions with Sp GpsB and the importance of its reduction or loss in S. pneumoniae . However, the observation that all three Δ pbp1a pbp2a deletion mutants were viable and both growth and morphology phenotypes were different between S. pneumoniae Δ pbp1a strains depleted for gpsB (Fig. 5d) and Δ pbp1a strains depleted for pbp 2a (Fig. 5e ) implies that Sp PBP2a binding is also just one function for Sp GpsB. It is possible that the Sp PBP2a:GpsB interaction is only part of the S. pneumoniae Δ gpsB phenotype and this interaction per se is not essential, unless the interaction of GpsB with an additional partner is also lost. Alternatively, since deleting the GpsB binding motif of Sp PBP2a did not abolish the interaction with GpsB completely, the deletion might reveal, or even generate, an unpredicted GpsB binding site, perhaps in the juxta-membrane region untouched by the deletions. Since the pbp2a mutant did not phenocopy gpsB depletion, and given the complex network of GpsB interactions in B. subtilis and L. monocytogenes , we also sought to extend the pneumococcal GpsB interactome starting from those proteins that were reported to form a complex with Sp GpsB by co-immunoprecipitation (co-IP) [24] . Besides the Sp GpsB interactions detected with Sp PBP2a and Sp MreC by BACTH, we also detected an interaction between Sp GpsB and the essential class B Sp PBP2x [44] (Supplementary Figure 6A ). Sp PBP2x, which contains a cytoplasmic domain abundant with arginines, also interacted with Sp GpsB in FP experiments (Supplementary Figure 6B ). However, a Sp GpsB: Sp PBP2x interaction was not detected by co-IP either using Sp GpsB-L-FLAG [3] as the bait and an anti-HA antibody to detect HA-tagged Sp PBP2x [24] or an anti- Sp PBP2x for native Sp PBP2x immnodetection, or Sp PBP2x-FLAG [3] as bait and an anti- Sp GpsB antibody for immunodetection of Sp GpsB (Supplementary Figure 6C ). These results suggest that Sp GpsB: Sp PBP2x complexes may be insufficiently abundant, or present only transiently, to be detected by co-IP in pneumococcal cells. Sp GpsB also interacted in BACTH with the class A Sp PBP1a (Supplementary Figure 6A ), which contains a LRLIKY motif in a putative helical region in its small cytoplasmic domain of 18 amino acids. On the other hand, no direct interaction was detected between Sp GpsB and Sp PBP2b either by BACTH (Supplementary Figure 6A ) or by FP (Supplementary Figure 6B ), consistent with the lack of any candidate GpsB-binding sequence motif in Sp PBP2b. The Sp PBP2b: Sp GpsB interaction detected previously by co-IP [24] (Supplementary Figure 6C ) is therefore likely to be indirect, presumably involving a bridging protein. The Sp GpsB Asp33Ala allele that resulted in a complete loss of binding to Sp PBP2a by FP (Supplementary Table 1 ) also abrogated interactions in BACTH with a markedly greater impact on interactions with Sp PBP2a compared to Sp MreC (Supplementary Figure 6A ). Sp GpsB Tyr23Ala and Sp GpsB Asp29Ala mutations had a greater impact on Sp MreC interactions than Sp GpsB Asp33Ala ; this pattern mirrors the impact of the equivalent mutations ( Lm GpsB Tyr27Ala , Lm GpsB Asp33Ala and Lm GpsB Asp37Ala ) on MreC interactions in L. monocytogenes (Supplementary Figure 3D ) and thus substantiates the evidence that different surfaces are used by GpsB to bind a specific class A PBP and MreC. Whilst the interactions of Sp GpsB with Sp EzrA and Sp StkP were confirmed by BACTH, and observed with the reciprocal hybrid pairs, they were unaffected by any of the Sp GpsB alleles mentioned above (Supplementary Figure 6A ). The interactions of GpsB in the pneumococcus, as detected by BACTH, FP and co-IP, are summarised in Supplementary Figure 6D . Taken as a whole, our data on three important bacterial systems agree that GpsB is an adaptor protein [29] , [30] , [31] that connects a major class A PG synthase with other cell wall and cell cycle proteins, and to cell shape determinants such as MreC. The identity and mode of interaction of the GpsB-binding partners varies from species to species and may reflect the different physiologies of each bacterium and their modes of growth and division. Bacterial cell growth and division necessitates tight co-ordination between the replication and segregation of the chromosome, the fission of the cell membrane and the remodelling of the PG. Consequently proteins and their complexes with major functions on either side of the membrane must co-ordinate their activities. One potential mechanism involves the interactions of major PG synthases with their intracellular regulators. Herein we present the first structures of the cell cycle adaptor, GpsB, in complex with the cytoplasmic mini-domains of PG synthases from three different bacteria, the rod-shaped B. subtilis and L. monocytogenes , in which gpsB is conditionally essential [11] , [12] , [19] and the ovococcal S. pneumoniae in which gpsB is essential [22] , [23] , [24] . In common with mammalian adaptors GGA [31] and 14-3-3 [45] proteins, the primary binding surface of GpsB is restricted to a conserved groove between α-helices The cytoplasmic mini-domains of the three PG synthases in the three organisms have little in common except that each utilises a conserved arginine in their respective sequences to interact with the cognate GpsB. The PG synthase arginine finger pokes into a negatively charged cavity situated between α-helices 1 and 2 of GpsB and is fixed in the same orientation in all structures, just as the phosphoryl group defines the binding orientation of peptides to 14-3-3 [45] . The arginine complements the cavity best when the mainchain amide protons of it and its downstream residue are accessible to form hydrogen bonds with Bs GpsB Asp35 , Lm GspB Asp37 or Sp GspB Asp33 . This scenario can occur when the arginine is either at the start of an α-helix, such as Bs PBP1 Arg8 , or at the i + 1 position in a type I β turn, such as Sp PBP2a Arg31 , which explains why free l -arginine does not displace pre-bound PBP peptides from GpsB even when present at 100-fold molar excess (Supplementary Figure 2E ). Similarly, contact to the backbone amide at the i + 2 position in 14-3-3 ligands is essential for binding [45] . Despite a lack of strong sequence and structural homology in the PG synthase cytoplasmic mini-domains, their binding is dependent upon an identical subset of GpsB residues including Bs GpsB Tyr25 , Bs GpsB Asp31 , Bs GpsB Asp35 (Fig. 1c ) and their structural equivalents Lm GspB Tyr27 , Lm GspB Asp33 , Lm GspB Asp37 (Fig. 2a ), and Sp GpsB Tyr23 , Sp GpsB Asp29 and Sp GspB Asp33 (Fig. 4c, d , Supplementary Figure 1A ). Mutations at these positions in GpsB from S. pneumoniae and L. monocytgenes are lethal or have marked growth defects (Fig. 5b, c ) [19] and do not interact with their cognate peptidoglycan synthase by FP (Supplementary Table 1 ) [19] or by BACTH (Fig. 5a ) [19] . A phenotype analysis of equivalent mutations in B. subtilis to assess their importance is not straightforward to determine for two reasons. First, a phenotype for the gpsB null mutant is only observed synthetically, when gpsB is mutated alongside either ftsA [12] or ezrA [11] . Second, a B. subtilis mutant lacking all class A PBPs is viable [46] , precluding an unequivocal assessment of the precise importance of the Bs GpsB: Bs PBP1 interaction. Nonetheless, the convergence of all our experimental data on three bacterial systems suggests strongly that the tyrosine and aspartate dyad also have important roles in B. subtilis . Furthermore, these amino acids are also conserved in the DivIVA/Wag31/antigen 84 actinobacterial homologues of GpsB, suggesting a role for them in recruiting cell wall synthesis enzymes to the hyphal tip and future branch sites [13] , [14] , regions that require nascent PG synthesis in filamentous bacteria. We originally set out to establish the common rules by which GpsB interacts with major PG synthases. Other than the arginine finger mode of GpsB recognition, we discovered how GpsB interacts with at least one class A PBP in each species; that Lm GpsB interacts with both the cell shape determinant, MreC [47] , and a regulator of Z-ring dynamics, EzrA [10] , while in S. pneumoniae we have confirmed the Sp GpsB:MreC interaction and newly identified interactions with the class A Sp PBP1a and with the essential class B Sp PBP2x [44] . These new data complement what was previously known about these interactions in B. subtilis [11] and S. pneumoniae [23] , [24] . How GpsB can interact with such disparate targets remains unknown but Bs GpsB Asp31 , Lm GpsB Asp33 and Sp GpsB Asp29 are important for interactions with PBPs and other proteins, including MreC, while Lm GpsB Asp37 and Sp GpsB Asp33 only interact with PBPs. There must be at least one other surface that is used by GpsB to form complexes with other proteins in its function as an adaptor. The GpsB:PBP interaction interface notably requires no more than three sidechains from any PBP to complex with GpsB. Protein:peptide contacts involving less well-conserved exosites that flank a small core, conserved peptide motif can contribute significantly to the affinity of protein:peptide interactions [48] , [49] , and the contribution of exosites to affinity, such as the juxta-membrane region, may explain why point mutations in Lm PBPA1 and Sp PBP2a have a significant impact using peptide fragments in vitro, but have reduced impact in bacterial cells. For instance, the Lm PBPA1 Arg8Ala mutation had negligible effect (Fig. 2c , Supplementary Figure 2D ) yet it reduced binding by > 15-fold (Supplementary Table 1 ). Similarly Sp PBP2a Arg31Lys,Arg33Lys had a > 25-fold impact on binding (Supplementary Table 1 ) yet growth phenotypes were not evident (Supplementary Table 2 ) until significant stretches of the cytoplasmic mini-domain were deleted (Supplementary Figure 5B ). We also found some differences in GpsB interactions between the species that may be related to GpsB species-specific function. In B. subtilis , we discovered a critical motif, SRxxR(R/K), found in close proximity to the membrane that could be used to predict novel GpsB partners. We used this information to identify an interaction network involving cell envelope binding and modifying proteins that most likely is underpinned by the GpsB hexamer. An RSxxxR motif was identified in class A PBPs from most streptococci and sequence features that could dictate GpsB-binding can be found in class A PBPs in other Gram-positive organisms such as the lactococci , Leuconostocaceae and enterococci, including the ESKAPE pathogen E. faecium (Supplementary Figure 7 ). However, sequence-based searches alone will not identify complete GpsB interactomes because the local structure of the sequence and its proximity to the membrane are also key parameters of GpsB binding. Sp PBP2a contains a partially conserved sequence RSxxxR (Supplementary Figure 4A ) that resembles the Bs PBP1 signature motif and the Sp PBP2a mini-domain interacts with each subunit of the Sp GpsB dimer in a different way (Fig. 4b–d ). We have observed here that mutation or deletion of the cytoplasmic mini-domain of Sp PBP2a does not phenocopy deletion or depletion of gpsB (Fig. 5c, e ). Similarly, a Δ pbpA1 strain did not phenocopy gpsB deletion in L. monocytogenes [19] . Taken together these results imply that there must be at least one other critical GpsB interaction partner, beyond respective class A PG synthases, that dictates its conditional essentiality in L. monocytogenes and B. subtilis , and essentiality under normal growth conditions in S. pneumoniae . In every Firmicute (and Actinobacterium) tested thus far, apart from S. aureus [26] , GpsB (or the homologous DivIVA/Wag31/antigen 84) acts as an adaptor to co-ordinate PG synthase activity with other processes depending on the physiology of the cell. GpsB hexamerisation can bridge the interaction of multiple binding partners, a function GpsB shares with 14-3-3 proteins that can form ternary complexes with BCR and Raf-1 by 14-3-3 dimerisation [50] . In bacilli, Bs GpsB plays a role in shuttling between the side wall during elongation and the septum during division [11] and, given that Bs PBP4b is regulated by σ factors E[35] and F[51], complexes of Bs PBP4b and Bs YrrS, bridged by Bs GpsB (Fig. 3c, d ), presumably play a role in the asymmetric cell division characteristic of endospore-forming bacilli. In listeria, which is closely related to bacilli and shares with them a rod-like morphology, GpsB appears to connect several PBPs with proteins with known roles in cytokinesis, including Z-ring polymerisation modulators (ZapA, EzrA, SepF), late division proteins (DivIB, DivIC) and the elongasome (MreC, MreBH) (Supplementary Figure 3C,D ), all of which except SepF and MreBH have also been tested in B. subtilis and found not to interact with Bs GpsB [11] . By contrast, S. aureus GpsB appears to modulate Z-ring assembly [26] , however, no interaction between FtsZ and GpsB has been identified in B. subtilis [11] , S. pneumoniae [23] , [24] or L. monocytogenes (Supplementary Figure 3C ). The pneumococci have an ovoid cell shape and lack key components such as the MinCD system for cell division site selection [52] , and MreB-like proteins required for side wall synthesis [53] . Presumably Sp GpsB interacts with one or more pneumococcal-specific proteins, the loss of which may be related to the lethal phenotype. Furthermore, Sp GpsB affects both StkP autophosphorylation [23] , [24] and the StkP-catalysed phosphorylation of Sp DivIVA [23] , [24] , Sp MapZ/LocZ [24] , [54] , Sp Jag/EloR/KhpB [55] , [56] , [57] and Sp MacP [58] . It is not yet clear how the complexes formed by these proteins are affected by their phosphorylation, except that Sp PBP2a activity is dependent upon phosphorylated Sp MacP [58] , at least in the presence of functional Sp StkP, or what the impact is of potential cross-talk to two-component signalling systems [59] . Finally, the different phenotypic outcomes associated with gpsB deletion or depletion in the three systems studied herein may reflect the presence of redundant systems in the large genome (4.2 Mbp) of the bacilli, partial redundancy in listeria (2.9 Mbp), and a relative absence of redundancy in the stripped-down genome (2.1 Mbp) of the pneumococci. The relative affinities and cellular concentrations of GpsB partners probably dictate which protein(s) is bound by GpsB at any point in a cell cycle-dependent manner; simultaneous interactions with multiple target proteins is likely to lead to an increase in avidity of GpsB [19] as commonly found in antibody:antigen interactions. However, the intricate networks involving GpsB will only be uncovered by validating the full GpsB interactome. Bacterial strains and growth conditions Supplementary Table 3 lists the bacterial strains used in this study. L. monocytogenes EGD-e-derived strains were routinely cultivated in brain heart infusion (BHI) broth or on BHI agar plates at 37 °C or 42 °C, where indicated. If required, erythromycin (5 µg −1 mL −1 ) and X-Gal (40–100 µg −1 mL −1 ) were added. All L. monocytogenes growth experiments were repeated three times and average values and standard deviations are shown. All S. pneumoniae strains were derived from unencapsulated serotype 2 D39 strains IU1824 (D39 Δ cps rpsL1 ) or IU1945 (D39 Δ cps ) [60] . S. pneumoniae strains were grown on Petri dishes containing the appropriate antibiotic, modified trypticase soy agar II (Becton-Dickinson) and 5% (vol per vol) defibrinated sheep blood (TSAII-BA), and the plates were incubated at 37 °C in 5% CO 2 . Bacteria were cultured statically in BHI (Becton-Dickinson) broth at 37 °C in an atmosphere of 5% CO 2 , and growth was monitored by OD 620 . Escherichia coli TOP10 and DH5α (lab stocks) were used as standard hosts for all cloning procedures [61] , and BL21(DE3) strains (lab stocks) were used for recombinant protein production. General methods, manipulation of DNA and oligonucleotide primers E. coli transformation and isolation of plasmid DNA (the plasmids used are listed in Supplementary Table 4 ) was performed according to standard protocols [61] . L. monocytogenes strains were transformed by electroporation. Enzymatic modification of plasmid DNA was carried out as described by the instructions given by the manufacturers. Quikchange mutagenesis was employed for restriction-free modification of plasmids [62] . DNA sequences of oligonucleotide primers are listed in Supplementary Tables 5 – 7 . All deletions and insertions were confirmed by PCR, and all constructs and clones were verified by Sanger DNA sequencing. Construction of L. monocytogenes mutant strains Plasmid pSH497 was first constructed to facilitate mutagenesis of the chromosomal copy of pbpA1 . A DNA fragment comprising recU and the first 2063 bp of pbpA1 was amplified from chromosomal DNA using primer pair SHW773/SHW774 and cloned into pMAD using Bam HI/ Nco I. An unwanted mutation in front of recU resulted in a correction of this plasmid by Quikchange with primer pair SHW777/SHW778. The corrected pSH497 was used as template in further Quikchange reactions to introduce Thr7Ala (SHW744/SHW745, pSH504), Arg8Ala (SHW746/SHW747, pSH505), Tyr11Ala (SHW755/SHW756, pSH506), Gln10Pro (SHW787/SHW788, pSH509) and Arg12Ala mutations (SHW748/SHW749, pSH507) into pbpA1 , or to remove pbpA1 nucleotides 4-1250 (SHW775/SHW776, pSH503). pSH508 ( pbpA1 Arg8Ala/Arg12Ala ) was obtained by Quikchange with primers SHW750/SHW751 and plasmid pSH505 as the template. An N-terminal fragment of pbpA1 was excised from the L. monocytogenes chromosome using plasmid pSH503 and the insertion/excision protocol for construction of clean deletions, resulting in strain LMS211. The mutated pbpA1 alleles present on pSH504-pSH509 were then reintroduced into LMS211 following the same protocol. L. monocytogenes fosfomycin susceptibility assays Fosfomycin susceptibility was recorded using filter discs (Ø 6 mm) soaked with 10 µL of a 10 mg −1 mL −1 fosfomycin solution. L. monocytogenes colonies, grown on BHI agar plates, were resuspended in BHI broth and used to swab-inoculate BHI agar plates. Filter discs soaked with fosfomycin were placed on top of the agar surface and the plates were incubated at 37 °C overnight. Diameter of growth inhibition zones was measured and corrected for the filter disc diameter. All experiments were performed three times and average values and standard deviations were calculated. Significance was determined using the t -test and differences were considered to be significant when P < 0.01. L. monocytogenes and B. subtilis BACTH assay The BACTH system [63] was used for analysis of protein:protein interactions. First, Lm GpsB was screened against Lm PBPA1 ( lmo1892 ) variants to identify residues in Lm PBPA1 that are important for binding Lm GpsB. To facilitate screening, we used a T25 fragment of Bordetella pertussis adenylate cyclase that had been fused to the N-terminal 91 amino acids of Lm PBPA1 to create a T25- Lm PBPA1 fusion containing the N-terminal cytoplasmic mini-domain and the transmembrane helix, but lacking lacking the extracellular glycosyltransferase and transpeptidase domains (T25-PBPA1ΔGT-TP) in plasmid pSH437 [21] . Lm PBPA1 residues that corresponded to the Bs GpsB binding motif of Bs PBP1 (Thr7, Arg8, Tyr11, Arg12) and additional positively charged amino acids (Lys14, Lys20, Lys21, Lys22, Lys25, Arg26, Lys28 and Arg29) in T25-PBP A1ΔGT-TP were replaced with alanine prior to screening against GpsB-T18. The pSH437 plasmid was mutated by Quikchange mutagenesis using the primer pairs SHW744/SHW754 (T7A, pSH485), SHW746/SHW747 (R8A, pSH486), SHW755/SHW756 (Y11A, pSH487), SHW748/SHW749 (R12A, pSH488), SHW757/SHW758 (K14A, pSH489), SHW759/SHW760 (K20A, pSH490), SHW761/SHW762 (K21A, pSH491), SHW763/SHW764 (K22A, pSH492), SHW765/SHW766 (K25A, pSH493), SHW767/SHW768 (R26A, pSH494), SHW769/SHW770 (K28A, pSH495) and SHW771/SHW772 (R29A, pSH496). pJR164 and pJR169 were constructed by cloning sepF (primers JR334/JR335 and Xba I/ Kpn I digestion) into pKT25 and p25-N, respectively. pJR165 and pJR170 were generated by cloning ezrA into pKT25 and p25-N, respectively, using primers JR339/JR340 and Xba I/ Kpn I for digestion. pJR172 and pJR174 were obtained by cloning zapA into pKT25 and p25-N, respectively, using primers JR337/JR338 and Pst I/ Kpn I. pJR213 was constructed by amplification of divIB with primers JR353/JR354 and cloning into pKT25 using Xba I/ Kpn I. pJR214 was generated by PCR amplification of divIC with primers JR355/JR356 and cloning into pKT25 using Xba I/ Kpn I. mreBH was amplified by PCR using oligonucleotides JR368/JR369 and cloned into pKT25 and p25-N using Xba I/ Kpn I, resulting in pJR233 and pJR236, respectively. pJR242 and pJR243 were obtained by cloning mreC into pKT25 and p25-N, respectively, using primers JR364/JR365 and Pst I/ Kpn I digestion. pbpA2 was cloned into pKT25 using oligonucleotides SHW153/SHW154 and Xba I/ Kpn I to create pJR250. pbpB1 was amplified with primers SHW157/SHW158 and cloned with Sma I/ Eco RI into pKT25, yielding pSH236. pbpB2 was amplified with primers SHW155/SHW156 and cloned into pKT25 after Pst I/ Bam HI digestion, yielding plasmid pSH235. pbpB3 was amplified using primers SHW159/160 and cloned by Pst I/ Bam HI digestion into pKT25, resulting in pSH237. Finally, pSH484 was obtained by removing the N-terminal domain from gpsB present on plasmid pSH226 in a PCR with the primer pair SHW752/SHW753. Plasmids encoding the respective genes fused to the N- or C-termini of the T18- or the T25-fragment of the Bordetella pertussis adenylate cyclase were co-transformed into E. coli BTH101. Transformants were selected on LB agar plates containing ampicillin (100 µg −1 mL −1 ), kanamycin (50 µg −1 mL −1 ), X-Gal (40 µg −1 mL −1 ) and IPTG (0.1 mM) and photographs were taken after 24 and 48h growth at 30 °C. The BACTH experiments in Fig. 2b and Supplementary Figure 3C, D were repeated at least twice. The same procedures outlined above were followed for the BACTH using B. subtilis GpsB except that co-transformants were grown on nutrient agar plates [11] , not LB, before imaging. These experiments were replicated reproducibly at least three times and a representative image is provided in Fig. 3c . Reciprocal tests for some interactions do not show the same results presumably because of the different expression levels for the individual fusion constructs as pKT25 is a low copy number plasmid whereas pUT18C is a high copy number plasmid. S. pneumoniae strain construction Mutant strains containing antibiotic resistance markers were constructed by transformation of CSP-1 induced competent pneumococcal cells with linear DNA amplicons synthesised by overlapping fusion PCR [64] . Mutant constructs were confirmed by PCR and DNA sequencing of chromosomal regions corresponding to the amplicon region used for transformation. Ectopic expression of wildtype gpsB with a Zn 2+ -inducible promoter (IU11286) was achieved by insertion into bgaA to create a Δ bgaA :: tet -P Zn - gpsB + construct using PCR-fused fragments. To investigate whether GpsB with allele changes of Y23A, V28A, D29A L32A D33A or I36A were functional, and given that gpsB is essential for the growth of S. pneumoniae D39, a merodiploid D39 Δ cps Δ gpsB < > aad9// Δ bgaA:: P Zn -gpsB + strain (IU11388) was constructed by transforming Δ gpsB < > aad9 into IU11286 in the presence of 0.5 mM ZnCl 2 + 0.05 mM MnSO 4 , which is required in the media to counteract the Zn 2+ toxicity [57] , [64] . For selection of gpsB alleles, a P c - erm cassette was fused to the 3ʹ end of gpsB with the desired mutations in the native chromosomal locus. The gpsB allele change-P c - erm amplicon was transformed into IU11388 in the presence of erythromycin and 0.5 mM ZnCl 2 + 0.05 mM MnSO 4 . The P c - erm cassette inserted at the 3ʹ end of gpsB + imparted no discernible growth phenotype compared to a wild-type strain (Fig. 5b ). The growth of merodiploid strain IU11388, and strains containing gpsB with allele changes complemented with ectopic expression of WT gpsB (IU12361, IU12363, IU12440, IU12612, IU12615, IU13121), or gpsB with allele changes linked to a FLAG tag complemented with ectopic expression of WT gpsB (IU13141, IU13364, IU13366, IU13368, IU13370, IU13372 and IU13374) were performed in the presence of 0.5 mM ZnCl 2 + 0.05 mM MnSO 4 . Transformation of ∆ pbp1a ::P c - erm into IU11388 (Δ gpsB <> aad9// Δ bgaA :: tet -P Zn - gpsB + ) and IU14365 ( ∆pbp2a markerless // Δ bgaA :: kan -P Zn - pbp2a + ) was performed in the presence of 0.4 mM ZnCl 2 + 0.04 mM MnSO 4 . Strains containing markerless pbp2a alleles in the native chromosomal locus were constructed using Janus cassette allele replacement [65] via an rpsL1 strain containing a ∆ pbp2a ::P c -[ kan - rpsL + ] construct (IU7853). Transformation of a Δ pbp1a amplicon into S. pneumoniae strains The function of the mutated pbp2a alleles was evaluated by transformations of 30 ng of a ∆ pbp1a ::P c - erm amplicon, obtained from strain E177 and containing ≈1 kb of flanking chromosomal DNA, into strains harbouring pbp2a mutations. Transformants were visualised after 24h incubation at 37 °C in 5% CO 2 . The numbers of colonies were normalised to 1 mL of transformation mixture. Growth and microscopy of S. pneumoniae strains Strains IU1945 (wild-type parent) and IU11286 ( gpsB + //Δ bgaA ::P Zn - gpsB + ) were inoculated from frozen glycerol stocks into BHI broth, serially diluted, and incubated for <13h statically at 37 °C in an atmosphere of 5% CO 2 . For IU11388 (∆ gpsB //Δ bgaA ::P Zn - gpsB + ) and all gpsB allele exchange strains complemented with bgaA ::P Zn - gpsB + , 0.5 mM ZnCl 2 + 0.05 mM MnSO 4 (+Zn) was added to BHI broth cultures to enable the ectopic expression of gpsB [64] . The next day, cultures at OD 620 ≈ 0.1–0.4 were diluted to OD 620 ≈ 0.003 in BHI broth lacking (−Zn) or containing (+Zn) 0.5 mM ZnCl 2 + 0.05 mM MnSO 4 and cultured under the same conditions. Growth was monitored turbidimetrically every 45 min to 1 h with a Genesys 2 spectrophotometer (Thermo Scientific). At 3.75 h after dilution into BHI broth with or without Zn/Mn supplement, cell pellets were obtained from 1 mL of culture, and resuspended in 100 µL of 4% paraformaldehyde. Cells were fixed for 15 min at RT and the tubes with fixed cells were left on ice until microscopy. For microscopic analyses, samples (1.5 μL) were taken and examined using a Nikon E-400 epifluorescence phase-contrast microscope. Growth and microscopy of strains containing pbp2a alleles were performed as above, but with no Zn/Mn addition to the BHI broth. Microscopy was performed at OD 620 ≈ 0.15. Growth and microscopy experiments of IU14381 ( ∆pbp2a// P Zn - pbp2a + ∆ pbp1a ) and IU14383 (Δ gpsB// P Zn - gpsB + ∆ pbp1a ) were performed as for IU11388 (∆ gpsB //P Zn - gpsB + ) except that overnight growths were carried out in BHI broth containing 0.2 mM ZnCl 2 + 0.02 mM MnSO 4 for IU14381, and 0.4 mM ZnCl 2 + 0.04 mM MnSO 4 for IU14383. Cultures were diluted into the same media as the overnight media for +Zn condition and into BHI broth without Zn/Mn for the −Zn condition. All growth measurements were reproducible and were repeated at least three times. The mean doubling time and the standard error of the mean ( ± ) are reported in Supplementary Figure 5B . Western blotting and immunodetection of S. pneumoniae strains To confirm the expression of gpsB with Y23A, V28A, D29A, L32A, D33A or I36A allele exchanges, western blot analyses were performed of strains constructed with gpsB -FLAG or gpsB variant-FLAG at the native site complemented by ectopic Zn-dependent expression of WT gpsB . 0.5 mM ZnCl 2 + 0.05 mM MnSO 4 (+Zn) was added to all BHI broth cultures to enable the ectopic expression of gpsB , and were diluted to OD 620 ≈ 0.003 and cultured under the same conditions to OD 620 ≈ 0.15 to 0.2. Under the +Zn condition, all FLAG-tagged gpsB allele exchange strains grew identically to WT gpsB + strain and to the untagged gpsB allele exchange strains. A parallel set of cultures was performed using BHI broth without addition of ZnCl 2 and MnSO 4 to confirm that FLAG-tagged gpsB allele strains grew identically to their untagged counterparts. Aliquots of 1.8 mL were centrifuged (5 min, 16,000 × g at 4 °C), and cell pellets were washed once with PBS. The supernatant was discarded and the pellets were frozen on dry ice for 5 min. The pellets were then thawed for 5 min at RT, resuspended in 80 µL of prewarmed 37 °C SEDS lysis buffer (0.1% deoxycholate, 150 mM NaCl, 0.2% SDS, 15 mM EDTA pH 8.0) [24] . Samples were incubated on a 37 °C shaking block at 300 rpm for 15 min, and were vortexed vigorously twice during the 15 min incubation. Total protein concentrations were determined using a Bio-Rad DC TM protein assay kit. 4 µg of total protein was loaded per lane on a 4–15% precast gradient SDS-PAGE gel (Bio-Rad), subjected to electrophoresis and transferred to a nitrocellulose membrane. FLAG-tagged GpsB proteins were detected with an anti‐FLAG rabbit polyclonal antibody (Sigma, F7425, 1:1400 dilution) as primary antibodies, and ECL anti-rabbit IgG horseradish peroxidase linked whole antibody as secondary (dilution 1:10,000). Chemiluminescent signals in protein bands were detected with an IVIS imaging system. MreC was detected with anti-MreC antibodies [66] by relabelling the nitrocellulose membrane after detection with anti-FLAG. Western detection of PBP2a in various PBP2a variant strains was performed essentially as above with exponentially growing cultures in BHI broth. 4 µg of total protein was loaded per lane onto a 10% precast SDS-PAGE gel (Bio-Rad). Electrophoresis was carried out for 1.5 h to allow separation of Sp PBP2a from a non-specific band. Anti- Sp PBP2a serum [67] was used at a dilution of 1:5000. The anti-serum against purified, recombinant Sp GpsB 1-63 was characterised by preparing lysates from gpsB + divIVA + WT (strain IU1945), Δ gpsB (IU6442) or Δ divIVA (IU8496) strains as described above. 4 μg of total protein was loaded per lane on a 4–20% precast gradient SDS-PAGE gel (Bio-Rad), and anti-GpsB serum from rabbit Ab-1432 was used at a dilution of 1:2000. Co-immunoprecipitation (Co-IP) of S. pneumoniae strains Co-IP experiments of S. pneumoniae FLAG-tagged strains were performed with the use of anti-FLAG magnetic beads [24] . Lysates were obtained from cultures grown exponentially at 37 °C in an atmosphere of 5% CO 2 in 400 mL of BHI to OD 620 ≈ 0.25–0.40 [24] . Cell pellets were washed once with 30 mL of 1X PBS (4 °C) and resuspended in 19.8 mL 1× PBS (4 °C). About 200 μL of 10% (vol per vol) paraformaldehyde solution (EMS) were added for crosslinking to a final concentration of 0.1% (vol per vol). Mixtures were incubated at 37 °C in an air incubator for 1 h. Cross‐linking reactions were quenched by the addition of 4 mL 1.0 M glycine followed by incubation at 25 °C for 10 min. Cells were collected by centrifugation (16,500 × g for 5 min at 4 °C). Pellets were washed once with 20 mL cold 1× PBS (4 °C) and resuspended in 2 mL of cold lysis buffer (50 mM Tris‐HCl pH 7.4, 150 mM NaCl, 1 mM EDTA, 1% Triton X100 (vol per vol)) with 1 tablet of protease inhibitor (ThermoFisher Scientific, 78429) freshly added per 10 mL of lysis buffer. The suspension was transferred into two lysing matrix B tubes (MP Biomedicals) with 1 mL in each tube. The tubes were shaken ten times in a FastPrep homogenizer (4×, 5 min on ice, 3×, 5 min on ice and 3×) with 6.0 M s −1 for 40 s each at 4 °C. Cell debris and lysing matrix from tubes were removed by centrifugation at 16,000 × g for 5 min at 4°C. The protein concentration of each sample was determined by Bio‐Rad DC TM protein assay (Bio‐Rad). About 1 mL of lysate with similar amounts of total protein (5–7 mg −1 mL −1 ) was added to tubes with 50 μL of anti‐FLAG magnetic beads (Sigma, M8823). The same amount of protein was loaded onto the beads for strains expressing FLAG‐tagged proteins and the corresponding control strains lacking FLAG‐tagged proteins in each experiment. The tubes were rotated for 2 h at 4 °C. The beads were washed three times with 1 mL of lysis buffer (4 °C) with 10 min incubation at 4 °C each time. FLAG‐tagged proteins were eluted from the beads by incubation with 100 μL of FLAG elution solution (150 ng 3X FLAG peptide per μL) (Sigma, F4799) for 30 min at 4 °C. A volume of 100 μL of the elution and of the original lysate added to magnetic beads (input) were separately mixed with 100 μL 2× Laemmli sample buffer (Bio‐Rad) containing 5% (vol per vol) β‐mercaptoethanol (Sigma) and heated at 95 °C for 1 h to break the cross‐links. A volume of 40 µL of each elution sample mixed with 2× sample buffer was loaded on each lane of a 4–15% precast SDS-PAGE gel and subjected to western blotting using affinity-purified Sp PBP2x polyclonal antibodies (dilution 1:10,000) [67] or an anti-GpsB antibody as the primary antibodies. S. pneumoniae BACTH assay The target genes were amplified by the PCR from S. pneumoniae D39 chromosomal DNA. PCR fragments for pbp2a, mreC, pbp1a , pbp2x and pbp2b were purified, digested with appropriate restriction enzymes and cloned into the corresponding sites of the pKT25/pUT18C vectors to generate plasmids encoding the corresponding hybrid proteins fused at the C-terminal ends of the T25 and T18 fragments, respectively. Plasmids pKNT25- gpsB /pUT18- gpsB , pKNT25- stkP /pUT18- stkP and pKNT25- ezrA /pUT18- ezrA were already constructed [24] . The mutated and truncated gpsB and pbp2a alleles were amplified from their respective DNA templates and the corresponding PCR products cloned into the corresponding sites of the BACTH vectors as described above for the wild-type alleles. E. coli DH5α transformants were selected on LB agar plates containing ampicillin (100 μg −1 mL −1 ) or kanamycin (50 μg −1 mL −1 ) and 0.4% glucose to repress leaky expression [63] . BACTH experiments, each pair of plasmids was co-transformed into the E. coli cya - strain BTH101 and co-transformation mixtures were spotted onto LB agar plates supplemented with ampicillin (100 mg −1 mL −1 ), kanamycin (50 mg −1 mL −1 ) and X-Gal (40 μg −1 mL −1 ), followed by incubation at 30 °C. Plates were inspected and photographed after 24 and 40 h. Plasmid pairs pKNT25/pUT18 and pKT25-zip/pUT18C-zip were used as negative and positive controls, respectively. All experiments were repeated at least twice. Plasmid construction for recombinant protein and peptide work (i) GpsB: All mutagenesis was undertaken by the Quikchange protocol; where mutagenesis reactions failed to generate a DNA fragment of the expected size, a modification of the Quikchange protocol with two separate PCR steps was used instead [69] . Glu17Ala, Asp31Ala and Asp35Ala mutations were introduced to the Bs GpsB 1-68 expression construct plasmid [19] by Quikchange. The Bs GpsB 5-64 construct was prepared by PCR amplification of gpsB from B. subtilis 168 genomic DNA using primers BsGpsB5start and BsGpsB64stop. The PCR product was ligated between the Nde I and Xho I sites of modified pET15b (M26L DJ-1 TEV site pET15b; gift from Mark Wilson, Addgene) with the nucleotides encoding the thrombin cleavage site replaced by a sequence encoding a TEV cleavage site. The Sp GpsB 1-63 expression construct (pET28 Sp GpsB 1-63 ) was prepared by PCR amplification of gpsB from S. pneumoniae R6 genomic DNA with primers SpGpsB5ndeI and SpGpsB3XhoI. This PCR product was ligated between the Nde I and Xho I sites of pET28a, and a stop codon was introduced by Quikchange mutagenesis in place of the codon for Pro64. The Sp GpsB 4-63 expression construct was generated in two steps; first the ORF encoding residues 1–63 of Sp GpsB was amplified with primers SpGpsBM11NcoI and SpGpsBM11XhoI using plasmid pET28 Sp GpsB 1-63 as the template. This DNA fragment was then ligated between the Nco I and Xho I sites of pET11M [70] before the codons for residues 1–3 of Sp GpsB were deleted by Quikchange mutagenesis with primers SpGpsB1to3del5 and SpGpsB1to3del3. (ii) PBP peptides; Ser16Cys, Ser7Ala, Arg8Ala, Ala10Pro, Arg11Ala and Arg28Ala mutations in Bs PBP1 1-32 fused to maltose binding protein (MBP) [19] were introduced by Quikchange mutagenesis. Plasmids expressing Lm PBPA1 1-20 and Sp PBP2a 23-45 peptides fused to MBP were prepared by PCR amplifying the relevant ORFs from L. monocytogenes strain EGD-e and S. pneumoniae R6 genomic DNA with primers Lm PBPA1ncoI5, Lm PBPA1xhoI3, Sp PBP2AncoI5 and SpPBP2AxhoI3, respectively. The subsequent PCR fragments were digested with Nco I and Xho I for ligating into similarly restricted pMAT11, a modified version of pHAT4 [70] . Ser19 and Lys21 in Lm PBPA1 were mutated in a single step by Quikchange to cysteine and stop codons, respectively; similarly Quikchange was used to change Sp PBP2a Gly43 and Arg46 to cysteine and stop codons, respectively. Further mutations in Lm PBPA1 were also made by Quikchange; the Arg8AlaSer16Arg double mutant was prepared in two successive steps with the Arg8Ala mutation made first, followed by Ser16Arg. The Sp PBP2x 1-29 construct was prepared in several steps. First, nucleotides 1–1165 of pbp2x were PCR amplified in two steps: an initial fragment generated from S. pneumoniae R6 genomic DNA with primers Sp PBP2x5/ Sp PBP2x3st1 was used as a template for further PCR amplification with Sp PBP2x5/ Sp PBP2x3st2 primers; this fragment was then ligated into the Nco I and Xho I sites of pMAT11. Second, cysteine, serine and stop codons were introduced by Quikchange in place of residues 30–32 with primers Sp PBP2xS30CL31SL32STOP5 and Sp PBP2xS30CL31SL32STOP3. A second Quikchange step (primers Sp PBP2xinsgly5, Sp PBP2xinsgly3) introduced extra codons encoding a GSG sequence after the TEV cleavage to improve cleavage of the MBP-PBP2x 1-29 fusion protein. (iii) YpbE and YrrS; The construct for expressing YpbE 130-240 was prepared in two steps; first, the ORF encoding residues 80-240 of YpbE was PCR amplified from genomic DNA and ligated between the Nde I and Xho I sites of pET28a. Second, the ORF encoding the N-terminal His-tag and residues 80–129 of YpbE was subsequently deleted by PCR amplification of the entire plasmid with primers YpbEtruncatencoi5 and YpbEtruncatencoi3, followed by Nco I restriction digestion and religation of the DNA with T4 DNA ligase. The construct for expressing YrrSΔ 13-16 was prepared by amplifying the yrrS gene from B. subtilis genomic DNA with flanking Nde I and Xho I sites and then ligating the PCR fragment between the same restriction sites in pET28a. The region coding for residues 13–16 of YrrS was subsequently deleted by Quikchange mutagenesis. Recombinant protein purification (i) GpsB; Bs GpsB 1-68 proteins used for FP assays were purified by Ni-NTA affinity chromatography followed by proteolytic removal of the His 6 -tag by thrombin and subsequent size exclusion chromatography [19] . The same protocol was used for Sp GpsB 1-63 except that an ammonium sulphate precipitation step was added after thrombin removal of the His 6 -tag. Ammonium sulphate was added to the thrombin-cleaved protein to a final concentration of 2.34 M (60% saturation at 0 °C) by adding a stock solution of 100% saturated ammonium sulphate that was prepared by adding solid ammonium sulphate directly to 50 mM Tris.HCl (pH 8), 300 mM NaCl, 10 mM imidazole. After stirring for 30 min at 4 °C the mixture was centrifuged at 19,000 × g for 20 min and solid ammonium sulphate then added to the supernatant to a final concentration of 2.8 M. After stirring at 4 °C for another 30 min the mixture was again centrifuged 19,000 × g for 20 min and further ammonium sulphate added to a final concentration of 3.5 M. After 30 min stirring the mixture was again centrifuged at 19,000 × g and the pellet resuspended in 10 mM Tris.HCl (pH 8), 250 mM NaCl before further purification by gel filtration [19] . Bs GpsB 5-64 , Bs GpsB 5-64 Lys32Glu and Sp GpsB 4-63 were expressed and purified by a similar protocol except that TEV protease, rather than thrombin, was used to remove the N-terminal His 6 -tag by overnight cleavage with TEV (1:50 ratio of TEV:GpsB) at 4 °C in a buffer of 50 mM Tris.HCl (pH 8.0), 300 mM NaCl, 250 mM imidazole, 1 mM DTT. The cleaved protein was then dialysed against 20 mM Tris.HCl (pH 8.0), 200 mM NaCl, 10 mM imidazole and manually passed over a 5 mL Ni-NTA superflow cartridge (Qiagen) to remove TEV and uncleaved proteins. The flow through from the column was concentrated and loaded onto a Superdex 75 XK16/60 (GE Healthcare) gel filtration column equilibrated in 10 mM HEPES.NaOH (pH 8.0), 100 mM NaCl. (ii) PBP peptides; The PBP peptides, generated as His-tagged MBP-fusion proteins, were purified by standard Ni-NTA affinity chromatography procedures [19] . The purified MBP-PBP fusions at 5 mg −1 mL −1 were fluorescently labelled in a buffer of 50 mM Tris.HCl (pH 7.0), 300 mM NaCl, 250 mM imidazole by mixing with either TAMRA-maleimide (Santa Cruz Biotechnology) or with fluorescein maleimide (Vector laboratories) to final concentrations of 625 μM and 1 mM from 25 and 40 mM stocks made in DMSO, respectively. After overnight incubation at 4 °C the labelling reaction was exchanged into a buffer of 10 mM Tris.HCl (pH 8.0), 250 mM NaCl, cleaved with TEV protease (1:50) and the labelled peptide separated from the MBP fusion partner by passing through a 3 kDa molecular mass cutoff centrifugal ultrafiltration device [19] . The Bs PBP1 1-17 , Lm PBPA1 1-15 and Sp PBP2a 27-40 peptides used for crystallisation and circular dichroism were synthesised chemically (Protein and Peptide Research Ltd, UK and Severn Biotech, UK). The fluorescein-labelled Bs YpbE 1-21 and Sp PBP2b 1-17 peptides used in FP assays were also synthesised chemically (Protein and Peptide Research Ltd); the Sp PBP2b 1-17 peptide encompasses the first seventeen amino acids of Sp PBP2b from strain R6, based on the annotated sequence in the NCBI database (accession NP_359110 ). (iii) BsPBP1 proteins; Recombinant Bs PBP1 proteins were purified from E. coli membrane pellets [19] resuspended in a buffer of 50 mM HEPES.NaOH pH 7.5, 500 mM NaCl, 3 mM MgCl 2 , 0.3 mM DTT supplemented with Roche complete EDTA-free protease inhibitor cocktail, lysozyme and DNAase. The lysate was clarified by centrifugation at 10,000 × g for 20 min and the supernatant centrifuged further for 1 h at 4 °C at 100,000 × g . The membrane pellet was resuspended in lysis buffer supplemented with 15% glycerol, 0.2 mM AEBSF, 0.5 mM DTT and Roche complete EDTA-free protease inhibitor. The resuspended membranes were ultracentrifuged for 1 h at 4 °C at 100,000 × g and the membrane pellet resuspended in resuspension buffer (50 mM HEPES.NaOH pH 7.5, 500 mM NaCl, 3 mM MgCl 2 , 2% reduced Triton X-100, 15% glycerol, 10 mM β-mercaptoethanol). After 2 h stirring at 4 °C the extract was ultracentrifuged at 100,000 × g for 30 min at 4 °C. The supernatant was supplemented with imidazole to 5 mM then incubated for 2 h at 4 °C with Sigma His select resin. This mixture was then passed through a gravity column and the resin washed with resuspension buffer supplemented with 5 mM imidazole and then Bs PBP1 proteins were eluted with resuspension buffer containing 250 mM imidazole. The His 6 -tag was removed by thrombin treatment, before the digest was purified by Superdex S200 size exclusion chromatography in a buffer of 10 mM HEPES.NaOH pH 7.5, 500 mM NaCl, 3 mM MgCl 2 , 0.1% reduced Triton X-100, 2% glycerol. Residual uncleaved Bs PBP1 proteins were removed by incubation with His select resin before concentraing and snap-freezing in liquid nitrogen. (iv) YpbE; The YpbE 130-240 protein and its S132C variant were expressed in BL21(DE3) cells by induction overnight at 17 °C with 0.5 mM IPTG when the culture had reached an optical density at 600 nm of 0.6. The cell pellet from a 2 L culture was resuspended in 70 mL of 50 mM Tris.HCl (pH 8), 10 mM NaCl, supplemented with 1 mL of 25× working concentration of Roche Complete EDTA free protease inhibitor cocktail and lysed by sonication. The lysate was then passed over a XK16 column packed with a 25 mL bed volume of Fast Flow Q-Sepharose and the flow through from the column then mixed with an equal volume of lysis buffer supplemented with saturated ammonium sulphate at room temperature. After 30 min stirring at 4 °C the mixture was centrifuged at 19,000 × g for 20 min and the supernatant mixed with saturated ammonium sulphate to a final concentration of 60%. This mixture was stirred for 30 min at 4 °C then centrifuged for 20 min at 19,000 × g . The supernatant was mixed further with ammonium sulphate to a final concentration of 80%. After 30 min stirring at 4 °C the mixture was centrifuged for 30 min at 19,000 × g then the pellet resuspended in 5 mL 10 mM MES buffer pH 6. The resuspended pellet was then loaded onto a 5 mL Fast Flow HiTrap SP column (GE Healthcare) equilibrated in 25 mM MES.NaOH pH 6 and the protein eluted with a linear gradient of 0–500 mM NaCl. Fractions containing YpbE 130-240 were pooled, concentrated and loaded onto a Superdex 75 XK16/60 gel filtration column (GE Healthcare) pre-equilibrated in PBS. (v) YrrS; YrrSΔ 13-16 was expressed in BL21(DE3) cells by overnight induction at 20 °C with 0.4 mM IPTG. The pellet from a 2 L culture was resuspended in 25 mL 50 mM Tris.HCl (pH 8), 500 mM NaCl supplemented with 0.5 mg −1 mL −1 lysozyme, 2 µg −1 mL −1 DNAase and Roche Complete protease inhibitor cocktail. The cell suspension was lysed by sonication, and centrifuged at 10,000 × g for 20 min at 4 °C to remove intact cells. The supernatant was centrifuged at 100,000 × g at 4 °C for 1 h and the membrane pellet was resuspended in 15 mL 50 mM Tris.HCl (pH 8), 500 mM NaCl 10% (vol per vol) glycerol and centrifuged again for 1 hr at 100,000 × g at 4 °C. The membrane pellet was frozen in liquid nitrogen and stored at −80 °C. The membrane pellet was resuspended in 10 mL of 50 mM Tris.HCl (pH 8), 500 mM NaCl, 2% reduced Triton X-100, 5 mM imidazole supplemented with Roche Complete EDTA free protease inhibitor cocktail. After 3 h gentle agitation at 4 °C the membrane suspension was centrifuged at 4 °C at 100,000 × g for 30 min. A 0.4 mL bed volume of Ni-NTA Sepharose (Qiagen) was added to the supernatant and mixed overnight at 4 °C in a tube roller before filtering through an empty gravity column. The Ni-NTA beads were washed three times with 4 mL of 50 mM Tris.HCl (pH 8), 500 mM NaCl, 0.1% reduced Triton X-100, 5 mM imidazole and YrrSΔ 13-16 was eluted from the column with 4 mL of the same buffer supplemented with 250 mM imidazole. The eluate was concentrated to 0.5 mL and loaded onto a Superdex 200 HR10/300 gel filtration column (GE Healthcare) equilibrated in 10 mM Tris.HCl (pH 8), 250 mM NaCl, 0.1% reduced Triton X-100. All recombinant proteins or peptides were concentrated and flash frozen in small aliquots in liquid nitrogen and stored at −80 °C. Crystallisation and structure determination Successful crystallisation of the N-terminal domains of GpsB proteins was improved by truncation of a few amino acids from both N- and C-termini, which are too far from the PBP binding site (25 and 45 Å, respectively) to affect binding and correspond to the minimum ordered portion of GpsB [19] . Co-crystallisation of Bs GpsB 5-64 : Bs PBP1 1-17 , Bs GpsB 5-64 Lys32Glu : Lm PBPA1 1-15 and Sp GpsB 4-63 : Sp PBP2a 27-40 followed the same procedure. Equal volumes of GpsB protein and PBP peptide, both in a buffer of 10 mM HEPES.NaOH (pH 8.0) and 100 mM NaCl, were mixed at final concentrations of 20 and 25 mg −1 mL −1 , respectively. This mixture, corresponding to a 1:5 molar ratio of protein:peptide, was subjected to sparse matrix crystallisation screening at room temperature with 100 nL drops dispensed by a Mosquito (TTP Labtech) liquid handling robot into 96 well MRC crystallisation plates. Unbound Sp GpsB 4-63 was crystallised by the same procedure, at the same protein concentration, except for the absence of added peptide. Crystals of Bs GpsB 5-64 : Bs PBP1 1-17 grew from 0.1 M HEPES/MOPS pH 7.5, 12.5% MPD, 12.5% PEG 1000 12.5% PEG 3350, 0.03 M MgCl 2 , 0.03 M CaCl 2 and were mounted in rayon loops and frozen directly in liquid nitrogen. Crystals of Bs GpsB 5-64 Lys32Glu : Lm PBPA1 1-15 grew from 0.1 M imidazole pH 8, 0.2 M zinc acetate, 20% PEG 3000 were transferred to a cryoprotectant comprising the well solution supplemented with 20% vol per vol PEG 300 and 2.5 mg −1 mL −1 of the Lm PBPA1 1-15 peptide; after 3 min the crystals were mounted in rayon loops and frozen in liquid nitrogen. The Sp GpsB 4-63 : Sp PBP2a 27-40 complex crystallised in 0.1 M Tris.HCl pH 8.5, 0.2 M lithium sulphate, 40% PEG400; crystals were mounted after 1 μL of the crystallisation mother liquor containing 2.5 mg −1 mL −1 Sp PBP2a 27-40 peptide was layered over the crystallisation drop immediately prior to freezing directly in liquid nitrogen. Crystals of unbound Sp GpsB 4-63 were obtained from 0.1 M Tris.HCl pH 8.5, 0.2 M magnesium chloride, 20% PEG 8000 and were cryoprotected by direct transfer to a solution of the mother liquor supplemented with 20% PEG400 before mounting and freezing as above. X-ray data were collected from crystals of unbound Sp GpsB 4-63 in house with a gallium METALJET TM (Bruker AXS GmbH) as X-ray source at a wavelength of 1.34 Å. All other diffraction data were collected at the DIAMOND synchrotron: for Bs GpsB 5-64 : Bs PBP1 1-17 data were collected on beamline I24 at a wavelength of 0.9686 Å; for Bs GpsB 5-64 Lys32Glu : Lm PBPA1 1-15 data were collected on beamline I04 at a wavelength of 0.9795 Å and for Sp GpsB 4-63 : Sp PBP2a 27-40 data were collected on beamline I03 at a wavelength of 0.9762 Å. For Bs GpsB 5-64 : Bs PBP1 1-17 and Sp GpsB 4-63 : Sp PBP2a 27-40 the diffraction images were indexed and integrated with XDS [71] and scaled with AIMLESS [72] . For Bs GpsB 5-64 Lys32Glu : Lm PBPA1 1-15 the diffraction images were indexed and integrated with DIALS [73] , scaled in XDS [71] and merged with AIMLESS [72] . For unbound Sp GpsB 4-63 the images were indexed, integrated, scaled and merged in Proteum 3 (Bruker AXS GmbH). For the three different GpsB:PBP complexes and the unbound Sp GpsB 4-63 the initial phases were obtained by molecular replacement (MR) in PHASER [74] . For Bs GpsB 5-64 : Bs PBP1 1-17 residues 5-64 from the structure of dimeric GpsB 1-68 (PDBid 4UG3 [19] ) were used as the search model for MR whereas for Bs GpsB 5-64 Lys32Glu : Lm PBPA1 1-15 the MR search model was the co-ordinates of the Bs GpsB 5-64 : Bs PBP1 1-17 complex with the peptide removed. For the unbound Sp GpsB 4-63 the search model for MR was the N-terminal domain of Lm GpsB (PDB code 4UG1 [19] ). For the Sp GpsB 4-63 : Sp PBP2a 27-40 complex, the co-ordinates of the unbound Sp GpsB 4-63 protein were used as a search model for MR. In all cases the molecular replacement solutions were visualised and rebuilt in COOT [75] . The Bs GpsB 5-64 Lys32Glu : Lm PBPA1 1-15 and Sp GpsB 4-63 : Sp PBP2a 27-40 complexes were refined in PHENIX.REFINE [76] while the Bs GpsB 5-64 : Bs PBP1 1-17 complex and unbound Sp GpsB 4-63 were refined using REFMAC [77] . The Ramachandran plot statistics (favoured/allowed) are: Bs GpsB 5-64 : Bs PBP1 1-17 100%/0%; Bs GpsB 5-64 Lys32Glu : Lm PBPA1 1-15 99.2%/0.8%; Sp GpsB 4-63 : Sp PBP2a 27-40 98.6%/1.4%, and unbound Sp GpsB 4-63 99.6%/0.4% allowed. Statistics for data collection and for the final refined models can be found in Table 1 . Representative electron density maps for the peptide-bound structures are displayed in stereographic mode in Supplementary Figure 8 . Table 1 Data collection and refinement statistics Full size table FP assays FP experiments were undertaken in a buffer of 10 mM Tris.HCl (pH 8.0), 250 mM NaCl, 0.1% reduced Triton X-100. The excitation wavelength was 540 nm and fluorescence emission was recorded above 590 nm for TAMRA-labelled peptides. The N-terminal domains of GpsB proteins Bs GpsB 1-68 , Lm GpsB 1-73 , Sp GpsB 1-63 were used in all experiments in preference to the full-length GpsB proteins due to the high solubility of the former, which facilitated achieving the high protein concentrations necessary to saturate peptide binding. The validity of the N-terminal domain as a substitute for full-length GpsB proteins in these experiments is supported by the comparable affinity of Bs GpsB and Bs GpsB 1-68 for a labelled Bs PBP1A 1-32 peptide in FP experiments (Supplementary Table 1 ). K d values ± the standard error, generated after simultaneously fitting all the binding data to a 1:1 interaction model are reported and there are three measurements at each data point in a titration. SPR All SPR experiments used a running buffer of 10 mM Tris.HCl (pH 8.0), 250 mM NaCl, 0.1% reduced Triton X-100. Bs PBP1 and Bs PBP1 17-914 were immobilised on the surface of a CM5 chip (GE Healthcare). For the Bs PBP1/YrrSΔ 13-16 titration 800 RUs of Bs PBP1 were immobilised on the chip surface; for the Bs PBP1/ Bs GpsB titration 1200 RUs of Bs PBP1 were immobilised. YrrSΔ 13-16 , which lacks residues 13–16 in the cytoplasmic domain, was used in these experiments to minimise non-specific interactions with the chip matrix; binding of YrrSΔ 13-16 to the reference surface was negligible and the deletion of residues 13–16 leaves the GpsB-binding motif intact. The YrrSΔ 13-16 titration was carried out in single-cycle mode, without regenerating the surface between successive injections of protein, because harsh reagents were necessary for full surface regeneration. The fit of the single-cycle mode data to a 1:1 binding model was achieved with a U -value of 2 and a corresponding χ 2 of 46.1. CD analysis CD spectra were recorded on a JASCO J-810 spectropolarimeter with a PTC-4235 Peltier temperature controller using 1 mm path length quartz cuvettes. For full wavelength scans a scan speed of 10 nm −1 min −1 and a response time of 4 s were used, the final spectra were the average of at least four measurements. Bs PBP1 1-32 CD spectra were recorded at 4 °C in a buffer of 20 mM sodium phosphate, pH 7.3 at a peptide concentration of 25 μM. Peptide helical contents were estimated from molar ellipticities at 222 nm using the equation helix = [ θ ] 222 nm / (39,500(1–2.57/ n )) [78] where n is the number of residues in the peptide. Lm PBPA1 1-15 CD spectra were analysed at 40 μM in 20 mM sodium phosphate buffer, pH 7.8, for samples containing 0, 40 and 60% trifluoroethanol (TFE). For samples containing 80% TFE, 5 mM sodium phosphate buffer, pH 7.8, was used. The CD spectra of Bs GpsB 1-68 proteins were measured at a concentration of 4.5 μM in a buffer of 20 mM sodium phosphate (pH 7.8) 150 mM NaCl. For thermal melt experiments, a response time of 8 s and scan rate of 1 °C −1 min −1 were used. All thermal melts were reversible as CD spectra recorded before and after the melts in the wavelength range 200–240 nm could be superimposed. Peptidoglycan pulldown assay PG pulldown assays were carried out in PBS buffer. B. subtilis PG (SigmaAldrich) was prepared as a 10 mg −1 mL −1 stock solution in PBS containing 0.02% sodium azide. 25 µg of protein were added to a 100 µL sample containing 66 µg of PG and the mixture incubated with gentle agitation at room temperature for 30 min. The mixture was centrifuged at 16,000 × g for 7 min, the supernatant removed and the pellet resuspended in 1 mL of ice-cold PBS and immediately centrifuged for 2 min at 16,000 × g . The pellet was resuspended in 1 mL of the appropriate buffer and centrifuged for 2 min at 16,000 × g . Finally the pellet was boiled for 3 min in 60 μL SDS-PAGE loading buffer before analysis by SDS-PAGE; the SDS-PAGE loading buffer lacked reducing agents for YpbE 130-240 Ser132Cys samples.